RETRACTED ARTICLE: AKT3-mediated IWS1 phosphorylation promotes the proliferation of EGFR-mutant lung adenocarcinomas through cell cycle-regulatedU2AF2RNA splicing AKT-phosphorylated IWS1 regulates alternative RNA splicing via a pathway that is active in lung cancer. RNA-seq studies in lung adenocarcinoma cells lacking phosphorylated IWS1, identified a exon 2-deficient U2AF2 splice variant. Here, we show that exon 2 inclusion in the U2AF2 mRNA is a cell cycle-dependent process that is regulated by LEDGF/SRSF1 splicing complexes, whose assembly is controlled by the IWS1 phosphorylation-dependent deposition of histone H3K36me3 marks in the body of target genes. The exon 2-deficient U2AF2 mRNA encodes a Serine-Arginine-Rich (RS) domain-deficient U2AF65, which is defective in CDCA5 pre-mRNA processing. This results in downregulation of the CDCA5 -encoded protein Sororin, a phosphorylation target and regulator of ERK, G2/M arrest and impaired cell proliferation and tumor growth. Analysis of human lung adenocarcinomas, confirmed activation of the pathway in EGFR -mutant tumors and showed that pathway activity correlates with tumor stage, histologic grade, metastasis, relapse after treatment, and poor prognosis. The higher complexity of the proteome relative to the genome is due to multiple factors, one of which is RNA splicing [1] . At least 97% of the genes in the human genome have introns [2] and more than 95% of them undergo alternative RNA splicing [3] . RNA splicing therefore plays a critical role in determining the biological phenotype [4] . Several additional observations also support the importance of alternative RNA splicing in biology. First, the pattern of alternative RNA splicing changes during differentiation and many of these changes contribute to the differentiation process and/or the phenotype of the differentiated cells [5] . In addition, cell survival and proliferation signals may function by regulating alternative RNA splicing [6] . Finally, changes in alternative RNA splicing caused by mutations in cis -acting regulatory elements, such as splicing enhancers or silencers, and changes in the expression and/or post-translational modification of RNA splicing regulators have been linked to the pathogenesis of several diseases, including cancer [7] , [8] , [9] . Two complementary molecular mechanisms may contribute to alternative RNA splicing, the rate of transcription and chromatin modifications in the body of transcribed genes. Splicing occurs cotranscriptionally and when the rate of transcription is high, it increases the probability for exons that are not efficiently spliced, to be spliced out of the mature transcript [10] . Also, chromatin modifications are recognized by readers of epigenetic marks, which form the nucleus for the assembly of molecular complexes that bind to, and functionally regulate RNA-associated enhancers or silencers of splicing, perhaps by altering the rate of assembly and the composition of spliceosomal complexes [11] , [12] , [13] . One cellular function, which interfaces with the RNA splicing machinery, is the cell cycle [14] . The connection between RNA splicing and the cell cycle was originally suggested by experiments in the yeast Saccharomyces cerevisiae , which showed that the impact of mutations in the cell cycle gene cdc5 , can be suppressed by removing the intron of the tubulin-encoding gene TUB1 [15] . Progression through the cell cycle depends on periodic changes of gene function, which can be achieved by multiple mechanisms, one of which is the periodic modulation of RNA splicing and spliceosomal components [14] . Importantly, some of the changes in RNA splicing are regulated by periodic shifts in the expression and/or the activity of known cell cycle regulators, such as the Aurora kinases [16] , the large RS domain-containing protein SON [17] , and the RNA-recognition motif (RRM)-containing proteins TgRRM1 [18] and CLK1 [14] . Despite the fact that a connection between RNA splicing and the regulation of the cell cycle has already been established, our understanding of the mechanisms and the consequences of RNA splicing during cell cycle progression, remains rudimentary. Exploring the links between RNA splicing and the cell cycle is likely to yield important information, with a significant impact in our understanding of human disease, especially cancer. Shifts in RNA splicing play an important role in many types of human cancer, including non-small-cell lung cancer (NSCLC) [19] , the second most common cancer, with more than 250,000 new cases per year in the United States. There are three NSCLC histological subtypes, adenocarcinomas, squamous cell carcinomas, and large-cell carcinomas [20] , and all of them carry a very poor prognosis with <5% survival in 5 years [21] . Following our original observations, linking the alternative RNA splicing of FGFR2 to the biology of NSCLC [22] , several additional shifts in alternative RNA splicing were described in these tumors. These include alternative RNA splicing shifts in the Bcl-X L , CD44, Androgen Receptor, HLA-G, and PKM genes. These shifts ultimately promote cell survival, metastasis, and chemoresistance, inhibit immune-surveillance mechanisms, or endow the cancer cells with a metabolic advantage [13] , [23] , [24] , [25] . Massive parallel exome and genome sequencing of 183 lung adenocarcinomas in one study, identified somatic mutations in the splicing factors U2AF1 and RBM10 and in several epigenetic factors, which may also regulate RNA splicing [26] . Such mutations may render the cancer cells vulnerable to modulators of the core splicing machinery, as suggested by experiments showing that H3B-8800, a recently described modulator of SF3B1, preferentially kills cancer cells with mutations in spliceosomal components. Mechanistically, H3B-8800 may function by promoting the retention of short GC-rich introns, in the mRNA of mutant cells [27] . Activating mutations in epidermal growth factor receptor ( EGFR ) and Kirsten rat sarcoma ( KRAS ) are the most common genetic alterations in NSCLC with 69% of the tumors harboring mutations in these genes. Both types of mutations activate multiple signaling pathways, including the AKT and the ERK pathways and both carry poor prognosis. Data in this report delineate a pathway, which regulates alternative RNA splicing in lung adenocarcinomas, and they show that the influence of the pathway on the biology of tumors harboring EGFR mutations is more robust, than its influence on the biology of tumors harboring KRAS mutations. We had previously shown that the transcription elongation factors IWS1 and AKT play a central role in the regulation of the alternative splicing of FGFR2 , by promoting the skipping of exon 8 from the mature FGFR2 mRNA transcript. The exclusion of the FGFR2 exon 8 depends on the phosphorylation of IWS1 by AKT (primarily AKT3) on Ser720/Thr721, which recruits SETD2 to an IWS1-containing complex in the C-terminal domain (CTD) of RNA polymerase II. This results in the trimethylation of histone H3 at K36 in the body of the transcribed FGFR2 gene, which triggers the skipping of exon 8 from the mature transcript. As a follow-up to this study, we proceeded to address the global effects of IWS1 and IWS1 phosphorylation in lung adenocarcinomas. To this end, we carried out an RNA-seq experiment in the lung adenocarcinoma cell line NCI-H522, in which IWS1 was either knocked down or replaced by its phosphorylation site mutant S720A/T721A. The results of this analysis revealed that exon inclusion was significantly more common than the exon skipping we observed with the FGFR2 gene. One of the genes undergoing exon inclusion was the U2AF2 gene, which encodes the core splicing factor U2AF65 [28] , [29] , [30] . Exon inclusion was also under the control of SETD2 and histone H3K36 trimethylation. However, the reader of the histone H3K36me3 mark was the p52 isoform of LEDGF [12] , which interacts with the RNA-binding protein SRSF1 [31] . Therefore, although the chromatin-modification mark promoting exon inclusion is the same as the mark promoting exon exclusion, the effector complexes assembled on H3K36me3 in the two cases are different. The alternatively spliced exon 2 encodes the U2AF65 N-terminal serine–arginine-rich domain (RS domain), which is required for the interaction between U2AF65 and the splicing cofactor Prp19 [32] , [33] , [34] , [35] . The binding of U2AF65 to Prp19 is required for RNA splicing and expression of a gene set, which includes CDCA5 , the gene encoding Sororin, a component of the cohesin complex [36] . Here, we show that the IWS1-regulated Sororin is phosphorylated by ERK and that phosphorylated Sororin promotes ERK phosphorylation. Remarkably, inhibition of the IWS1 phosphorylation pathway, which regulates the Sororin/ERK positive feedback loop, results in inhibition of ERK phosphorylation, even in tumors with activating KRAS or EGFR mutations. The Sororin/ERK feedback loop described above, promotes the expression of CDK1 and CCNB1 (Cyclin B1), and the progression through the G2/M phase of the cell cycle. Importantly, similar to other cell cycle-regulatory pathways, the IWS1 phosphorylation pathway is also cell cycle-regulated. Mouse xenograft experiments confirmed that the IWS1 phosphorylation-dependent U2AF2 mRNA splicing controls tumor growth in vivo. Moreover, our studies on human lung adenocarcinoma samples and our analyses of the data on lung adenocarcinomas in publicly available datasets, confirmed the activation of the IWS1 phosphorylation pathway in these tumors. More important, the data derived from these studies also showed that the activity of this pathway correlates with tumor grade, stage, metastatic potential, relapse after treatment, and reduced patient survival, in patients with tumors harboring activating EGFR , but not KRAS mutations. This observation was in agreement with our data showing that tumor cell lines with EGFR mutations exhibit a stronger dependence on this pathway than tumor cell lines with KRAS mutations. Overall, the data in this report describe a pathway, which starts with the phosphorylation of IWS1 by AKT3 and results in the modulation of cell-cycle progression. The importance of this pathway to human cancer was confirmed by our studies on human lung adenocarcinomas and by meta-analysis of pre-existing patient data. IWS1 expression and phosphorylation regulate alternative mRNA splicing We had previously reported that IWS1 phosphorylation at Ser720/Thr721, primarily by AKT3, resulted in the exclusion of exon 8 from the FGFR2 mRNA in the human NSCLC cell lines NCI-H522 and NCI-H1299 [22] . To explore the molecular mechanisms driving IWS1 phosphorylation-regulated RNA splicing and gene expression, we examined the transcriptome of shControl, shIWS1, shIWS1/wild-type IWS1 rescue (shIWS1/WT-R), and shIWS1/IWS1S720A/T721A rescue (shIWS1/MT-R) NCI-H522 cells by RNA-Seq. This allowed us to identify additional target genes of the IWS1 phosphorylation pathway. First, we confirmed the downregulation of IWS1 in cells transduced with the lentiviral shIWS1 construct and the rescue of IWS1 expression in shIWS1-transduced cells with Flag-tagged wild-type IWS1, or the mutant IWS1-S720A/T721A (Fig. 1a ). Analysis of the RNA-seq data, identified 1621 genes, differentially expressed between shControl and shIWS1 cells and 562 genes differentially expressed between shIWS1/WT-R and shIWS1/MT-R cells ( p ≤ 0.01, FDR ≤ 0.2). Three hundred and forty genes upregulated or downregulated in shIWS1 cells were similarly upregulated or downregulated in shIWS1/MT-R cells (Supplementary Fig. 1a, b ). Moreover, 19 out of the FDR-ranked top 100 differentially expressed genes, in shControl vs shIWS1 cells, were also differentially expressed in shIWS1/WT-R versus shIWS1/MT-R cells (Supplementary Fig. 1c ). Gene-set enrichment analysis of differentially expressed genes [37] revealed significant enrichment of genes involved in RNA metabolism and the regulation of RNA processing (Supplementary Fig. 1d ). Fig. 1: IWS1 expression and/or phosphorylation regulate alternative mRNA splicing. a Western blots of NCI-H522 and NCI-H1299 cell lysates, transduced and probed with the indicated constructs and antibodies. b Overlaps between differentially-expressed and differentially spliced genes in the indicated groups ( q < 0.05). c Bar graphs of alternative splicing events with exon inclusion. The comparisons were limited to alternative splicing events with a percentage of the alternatively spliced exon spliced in (psi/ψ) >0.6 and a p value < 0.05. d GO analysis of statistically significant alternative splicing events in the indicated groups ( p < 0.05). Red boxes highlight gene sets involved in the regulation of RNA processing. e Volcano plots of all the exon inclusion and exclusion alternative splicing events, detected by DEXseq in the indicated groups. The statistically significant events ( p < 0.05) with a percentage spliced in (psi/ψ) level of >0.6 or <0.4 are shown in red. Statistically significant events in the GO functions RNA splicing or RNA metabolic processes are shown in green. Alternatively spliced IWS1 targets validated in this report are shown in blue. f (Upper panel) RT-PCR of U2AF2 in the indicated NCI-H522 and NCI-H1299 cells, using primers mapping in exons 1 and 3, 3 and 5, and 8 and 10 (control). GAPDH was used as the loading control. The U2AF2 E2/E3 ratio was calculated from the GAPDH-normalized levels of the RT-PCR products. The bars show the mean ratio ± SD in the indicated NCI-H522 and NCI-H1299 cells relative to shControl. g Sequencing chromatograms of the two alternatively spliced U2AF2 RNA transcripts. h (Upper) UCSC browser snapshot showing exons 1, 2, and 3 of the human U2AF2 gene. The map position of the PCR primer sets used in the ChIP experiments in this figure is indicated by blue marks. (Lower) ChIP assays of IWS1 on the U2AF2 and GAPDH genes in shControl, shIWS1 shIWS1/WT-R and shIWS1/MT-R NCI-H522 and NCI-H1299 cells. Bars show the mean fold enrichment (anti-IWS1 IP, vs IgG control IP) in IWS1 binding, in shIWS1 relative to shControl cells or in shIWS1/MT-R relative to shIWS1/WT-R cells ±SD. Data were normalized relative to the input (2%). All assays were done in triplicate, on three biological replicates. n.s: non-significant, * p < 0.05, ** p < 0.01, *** p < 0.001, **** p < 0.0001 (one-sided unpaired t -test). Full size image Analysis of the data for differential exon usage, by DEXseq [38] identified 1434 differentially employed exons (corresponding to 851 genes) between shControl and shIWS1 cells and 436 differentially employed exons (corresponding to 273 genes) between shIWS1/WT-R and shIWS1/MT-R cells (FDR ≤ 0.05). The 1796 differentially expressed genes and the 692 genes with differential exon usage in shIWS1 versus shControl cells exhibited an overlap of 165 genes ( p ≤ 0.05). Similarly, the 858 differentially expressed genes and the 230 genes with differential exon usage, between shIWS1/MT-R and shIWS/WT-R cells, revealed an overlap of 44 genes (Fig. 1b ). Exon inclusion and exon skipping represent common alternative RNA-splicing events. Our earlier studies had linked IWS1 phosphorylation with an exon skipping event in the FGFR2 gene [22] . Here, we analyzed the exon usage data in both shIWS1 versus shControl and shIWS1/WT-R versus shIWS1/MT-R cells, and we observed that the most common event associated with the expression and phosphorylation of IWS1, was exon inclusion (Fig. 1c ). GO (Gene Ontology)–biological process-based functional analyses of the alternative splicing events in shControl versus shIWS1 and shIWS1/WT-R versus shIWS1/MT-R cells identified GO functions “RNA splicing” and “RNA metabolic process”, among the top functions regulated by IWS1 expression and phosphorylation (Fig. 1d, e ). Comparisons were limited to alternative splicing events whose abundance changed significantly with the expression and phosphorylation of IWS1 ( p < 0.05). These findings imply that the effect of IWS1 on RNA processing may be direct or indirect. The indirect effect may be due to the IWS1 expression and phosphorylation-dependent differential regulation of genes involved in RNA processing. Validation of the RNA-seq data, using RT-PCR, confirmed several IWS1 and IWS1 phosphorylation-regulated alternative RNA-splicing events, characterized by exon inclusion (Fig. 1 and Supplementary Fig. 1g–j ). One of these events is the inclusion of exon 2 in the mature mRNA transcript of U2AF2 , the gene encoding the splicing factor U2AF65. Whereas the predominant U2AF2 mRNA transcript in shControl and shIWS1/WT-R cells contains exon 2, the predominant transcript in shIWS1 and shIWS1/MT-R cells is a transcript lacking exon 2 (Fig. 1f , g). The decrease in the E2/E3 ratio in shIWS1 and shIWS1/MT-R, relative to shControl cells, and the rescue of the shIWS1 phenotype by wild-type IWS1, were confirmed by quantitative RT-PCR (Supplementary Fig. 1e upper panels). Importantly, the knockdown of IWS1 and the rescue with the IWS1-S720A/T721A mutant did not significantly change the expression of U2AF2 or the inclusion of the U2AF2 exon 3 in NCI-H522 and NCI-H1299 cells (Supplementary Fig. 1f , upper panel) (Supplementary Fig. 1f , lower panel). In parallel experiments, we examined the alternative RNA splicing of FGFR2 in the same cells, by qRT-PCR. The results showed that the IIIb/IIIc FGFR2 transcript ratio was increased in shIWS1 and shIWS1/MT-R cells (Supplementary Fig. 1e , lower panel), confirming our earlier findings [22] . The preceding findings showed that the inclusion of exon 2 in the U2AF2 mRNA depends on IWS1 phosphorylation, and suggested that the shift in U2AF2 mRNA splicing caused by the knockdown of IWS1 in NCI-H522 and NCI-H1299 cells might be rescued by the phosphomimetic mutant IWS1-S720D/T721E (DE MT-R) (Fig. 1a ). Expression of this mutant in shIWS1-transduced cells indeed rescued the phenotype and confirmed the critical role of IWS1 phosphorylation in this process (Supplementary Fig. 1f , e, upper panel). To determine whether IWS1 is directly involved in U2AF2 mRNA splicing, we used chromatin immunoprecipitation (ChIP) to examine the binding of IWS1 to the U2AF2 exons 2 and 3 in shControl, shIWS1, shIWS1-WT-R, shIWS1-MT-R NCI-H522, and NCI-H1299 cells. The results revealed that IWS1 binds exons 2 and 3 of U2AF2 , suggesting its direct involvement to the U2AF2 alternative RNA splicing (Fig. 1h ). IWS1 WT and IWS1-S720A/T721A bind equally well (Fig. 1h ), suggesting that IWS1 phosphorylation controls U2AF2 exon 2 alternative RNA splicing by regulating events occurring after the binding of IWS1 to chromatin. IWS1 phosphorylation-dependent mRNA splicing of U2AF2 is regulated by serum and IGF1 via AKT3 IWS1 is phosphorylated by AKT3 and to a lesser extent by AKT1 at Ser720/Thr721 [22] . To determine the physiological significance of this observation, we examined whether IGF1 stimulation of serum-starved NCI-H522 and NCI-H1299 cells promotes U2AF2 exon 2 inclusion along with the expected AKT activation and IWS1 phosphorylation. In addition, we examined whether IGF1 enhances the skipping of the FGFR2 exon 8, increasing the ratio of IIIb/IIIc FGFR2 transcripts. The results confirmed that both the inclusion of exon 2 in the U2AF2 transcripts and the skipping of FGFR2 exon 8, indeed parallel the activation of AKT (Fig. 2a , Supplementary Fig. 2a ). To address whether the U2AF2 exon 2 inclusion depends on AKT activation, we treated NCI-H522 and NCI-H1299 cells growing in serum-containing media with 5 μM of the AKT inhibitor MK2206. The results confirmed that at this concentration, which fully inhibits all AKT isoforms, MK2206 inhibits both AKT and IWS1 phosphorylation and U2AF2 exon 2 inclusion (Fig. 2b , Supplementary Fig 2b , upper panels). 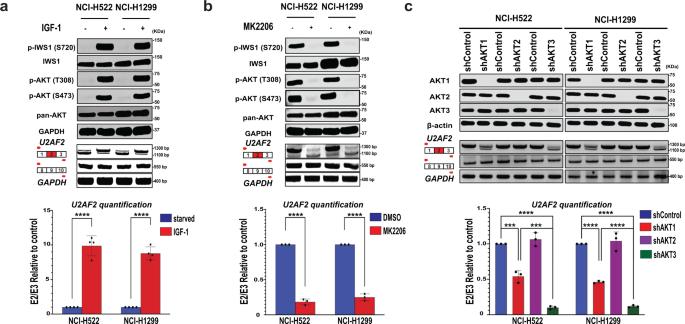Fig. 2: IWS1 phosphorylation-dependent mRNA splicing ofU2AF2is regulated by serum and IGF-1-induced signals, transduced by AKT3. a(Upper panel) Following serum starvation for 24 h, NCI-H522 and NC-H1299 cells were stimulated with IGF-1 or harvested. Four hours later, the stimulated cells were lysed and all the lysates were probed with the indicated antibodies. (Middle panel) RT-PCR with mRNA derived from the cells shown in the upper panel and oligonucleotide primers mapping to exons 1 and 3 of theU2AF2gene (Lower panel) TheU2AF2geneE2/E3ratio was calculated following quantification of the RT-PCR products in the middle panel. The bars show this ratio (mean± SD) in IGF1-stimulated and in unstimulated, serum-starved NCI-H522 and NCI-H1299 cells.b(Upper panel) Lysates of NCI-H522 and NCI-H1299 cells, treated with MK2206 (5μM) or DMSO for 4 h, were probed with the indicated antibodies. (Middle panel) RT-PCR reactions, using mRNA derived from the cells in the upper panel and oligonucleotide primers mapping inU2AF2exons 1 and 3. (Lower panel) TheU2AF2mRNAE2/E3ratio was calculated following quantification of the RT-PCR products in the middle panel. The bars show this ratio (mean± SD) in MK2206-treated (5μM) and in DMSO-treated NCI-H522 and NCI-H1299 cells.c(Upper panel) Lysates of NCI-H522 and NCI-H1299 cells, transduced with shControl, shAKT1, shAKT2, or shAKT3, were probed with the indicated antibodies. (Middle panel) RT-PCR reactions, using mRNA derived from the cells in the upper panel and oligonucleotide primers mapping inU2AF2exons 1 and 3 show that knocking down AKT3, and to a lesser extent AKT1, inhibits the inclusion of exon 2 in matureU2AF2mRNA transcripts in both cell lines. (Lower panel) TheU2AF2 E2/E3ratio was calculated following quantification of the RT-PCR products in the middle panel. The bars show this ratio (mean ± SD) in shControl, shAKT1, shAKT2 and shAKT3 NCI-H522 and NCI-H1299 cells. All experiments in this figure were done in triplicate, on three biological replicates. n.s: non-significant, *p< 0.05, **p< 0.01, ***p< 0.001, ****p< 0.0001 (one-sided unpairedt-test). The same treatment also increased the relative abundance of the exon 8-containing IIIb transcript of FGFR2 (Supplementary Fig. 2b lower panel), as expected. To determine whether it is the AKT3 isoform of AKT, which is responsible for these shifts in alternative RNA splicing, we transduced NCI-H522 and NCI-H1299 cells with shControl, shAKT1, shAKT2, or shAKT3 lentiviral constructs, and we examined the effects of the transduction on the alternative RNA of splicing of U2AF2 and FGFR2 . The results (Fig. 2c , Supplementary Fig. 2c ) confirmed that only the knockdown of AKT1 and AKT3 phenocopies the MK2206 results and that the effect of the AKT3 knockdown is significantly more robust than the effect of the AKT1 knockdown. These findings are consistent with the phosphorylation of IWS1 primarily by AKT3, and strongly support the hypothesis that the phosphorylation of IWS1, primarily by AKT3 and secondarily by AKT1, plays an important role in the physiological regulation of alternative RNA splicing by external signals. Fig. 2: IWS1 phosphorylation-dependent mRNA splicing of U2AF2 is regulated by serum and IGF-1-induced signals, transduced by AKT3. a (Upper panel) Following serum starvation for 24 h, NCI-H522 and NC-H1299 cells were stimulated with IGF-1 or harvested. Four hours later, the stimulated cells were lysed and all the lysates were probed with the indicated antibodies. (Middle panel) RT-PCR with mRNA derived from the cells shown in the upper panel and oligonucleotide primers mapping to exons 1 and 3 of the U2AF2 gene (Lower panel) The U2AF2 gene E2/E3 ratio was calculated following quantification of the RT-PCR products in the middle panel. The bars show this ratio (mean± SD) in IGF1-stimulated and in unstimulated, serum-starved NCI-H522 and NCI-H1299 cells. b (Upper panel) Lysates of NCI-H522 and NCI-H1299 cells, treated with MK2206 (5μM) or DMSO for 4 h, were probed with the indicated antibodies. (Middle panel) RT-PCR reactions, using mRNA derived from the cells in the upper panel and oligonucleotide primers mapping in U2AF2 exons 1 and 3. (Lower panel) The U2AF2 mRNA E2/E3 ratio was calculated following quantification of the RT-PCR products in the middle panel. The bars show this ratio (mean± SD) in MK2206-treated (5μM) and in DMSO-treated NCI-H522 and NCI-H1299 cells. c (Upper panel) Lysates of NCI-H522 and NCI-H1299 cells, transduced with shControl, shAKT1, shAKT2, or shAKT3, were probed with the indicated antibodies. (Middle panel) RT-PCR reactions, using mRNA derived from the cells in the upper panel and oligonucleotide primers mapping in U2AF2 exons 1 and 3 show that knocking down AKT3, and to a lesser extent AKT1, inhibits the inclusion of exon 2 in mature U2AF2 mRNA transcripts in both cell lines. (Lower panel) The U2AF2 E2/E3 ratio was calculated following quantification of the RT-PCR products in the middle panel. The bars show this ratio (mean ± SD) in shControl, shAKT1, shAKT2 and shAKT3 NCI-H522 and NCI-H1299 cells. All experiments in this figure were done in triplicate, on three biological replicates. n.s: non-significant, * p < 0.05, ** p < 0.01, *** p < 0.001, **** p < 0.0001 (one-sided unpaired t -test). Full size image U2AF2 exon 2 inclusion, induced by IWS1 phosphorylation at Ser720/Thr721, depends on histone H3K36 trimethylation by SETD2 We had previously reported that IWS1 phosphorylation by AKT3 promotes the exclusion of exon 8 from the mature FGFR2 mRNA transcript, via a process that depends on histone H3K36 trimethylation by SETD2, and that the latter is recruited to the CTD of RNA Pol lI by phosphorylated IWS1 [22] . To determine whether the U2AF2 exon 2 inclusion phenotype also depends on histone H3K36 trimethylation, we performed ChIP assays in shControl, shIWS1, shIWS1/WT-R, and shIWS1/MT-R NCI-H522 and NCI-H1299 cells, addressing the abundance of H3K36me3 marks on exons 2 and 3 of U2AF2 . The U2AF2 transcriptional start site (TSS) and the GAPDH gene, as well as exons 8 and 9 of FGFR2 , were used as controls. The results confirmed the IWS1 phosphorylation-dependent trimethylation of histone H3 at K36, in exons 8 and 9 of the FGFR2 gene (Supplementary Fig. 3a ). In addition, they showed that the IWS1 phosphorylation-dependent U2AF2 exon 2 inclusion is also associated with the trimethylation of histone H3 at K36 in U2AF2 exons 2 and 3 (Fig. 3a ). In parallel experiments, the AKT inhibitor MK2206 phenocopied the phosphorylation-site mutant of IWS1 (Fig. 3b ), confirming that H3K36 trimethylation in U2AF2 exons 2 and 3 was due to IWS1 phosphorylation by AKT. Given the importance of SETD2 on transcription-coupled H3K36 trimethylation, we used ChIP assays to also address the binding of SETD2 to exons 2 and 3 of U2AF2 , in NCI-H522 and NCI-H1299 cells transduced with a lentiviral construct of hemagglutinin (HA)-tagged SETD2 (HA-SETD2). The TSS of U2AF2 GAPDH gene and exons 8 and 9 of FGFR2 were again used as controls. The results revealed that the pattern of SETD2 binding parallels the abundance of H3K36me3 marks in both exons 2 and 3 of U2AF2 (Fig. 3c ) and exons 8 and 9 of FGFR2 (Supplementary Fig. 3b ). These data combined suggest that the IWS1 phosphorylation-dependent histone H3K36 trimethylation is mediated by SETD2. Fig. 3: U2AF2 Exon 2 inclusion, induced by IWS1 phosphorylation at Ser720/Thr721, depends on H3K36 trimethylation by SETD2. a ChIP assays showing the abundance of H3K36me3 in the indicated NCI-H522 (left) and NCI-H1299 (right) cells. Bars show the mean fold enrichment in H3K36me3 (anti-H3K36me3 IP, vs IgG control IP) in the indicated regions of the U2AF2 gene, in shControl, shIWS1, shIWS1/WT-R and shIWS1/MT-R cells ±SD. Data were normalized relative to the input (2%). b ChIP assays showing the abundance of H3K36me3 in the indicated NCI-H522 (left) and NCI-H1299 (right) cells, treated with MK2206 (5μM) or DMSO. The bars show the mean fold enrichment of H3K36me3 (anti-H3K36me3 IP, vs IgG control IP) in the indicated regions of the U2AF2 gene, ±SD. Data were normalized relative to the input (2%). c ChIP assays showing the binding of HA-SETD2 in the indicated NCI-H522 (left) and NCI-H1299 (right) cells, transduced with a lentiviral HA-SETD2 construct. The bars show the mean fold enrichment in SETD2 binding (anti-HA IP, vs IgG control IP) ±SD. Data were normalized relative to the input (2%). The expression of HA-SETD2 is shown in Supplementary figure 4a. d (Upper panel) Lysates of NCI-H522 (left) and NCI-H1299 (right) cells transduced with the indicated constructs, were probed with the antibodies, as shown. RT-PCR addressing U2AF2 exon 2 splicing in the same cells. (Middle panel) GAPDH -normalized E2 and E3 bands in the RT-PCR experiment above, were used to calculate the E2/E3 ratio±SD. (Lower panel) Ratio of the U2AF2 exons 2 and 3 levels in the same cells ±SD, as determined by quantitative RT-PCR. E2/E3 ratio is shown relative to shControl (value = 1). All experiments had three biological replicates, all done in triplicate. n.s non-significant, * p < 0.05, ** p < 0.01, *** p < 0.001, **** p < 0.0001 (one-sided unpaired t -test). e Snapshots of the integrative genomic viewer showing the ChIP-Seq-determined distribution of Flag-IWS1, HA-SETD2, and histone H3K36me3, in U2AF2 . Parallel snapshots show the distribution of RNA reads in the RNA-seq experiment. Scale represents reads per million (RPM). Snapshots of peaks detected in the two biological replicates are shown. Black box highlights U2AF2 exons 2, 3 and adjacent regions. Full size image The preceding data suggested that the enzymatically active SETD2 contributes to the IWS1 phosphorylation-dependent regulation of the U2AF2 alternative RNA splicing. To determine whether it is also required, we knocked down SETD2 in NCI-H522 and NCI-H1299 cells and we rescued the knockdown with wild-type SETD2 or the SETD2 methyltransferase mutant R1625C [39] . Using RT-PCR and qRT-PCR, we observed that the knockdown of SETD2 phenocopies the knockdown of IWS1 on the splicing of the U2AF2 and FGFR2 mRNAs and that the effect of the knockdown on both the U2AF2 and FGFR2 mRNA splicing is rescued by the wild-type SETD2, but not by its methyltransferase mutant (Fig. 3d , Supplementary Fig. 3c ). We conclude that the enzymatic activity of SETD2 is indeed required for the regulation of the alternative splicing of both the U2AF2 and FGFR2 mRNAs. If SETD2 is recruited to the CTD of RNA Pol II by phosphorylated IWS1, wild-type SETD2 should not rescue the shIWS1 and shIWS1/MT-R phenotype. This was confirmed by experiments addressing the rescue of U2AF2 RNA splicing in shControl, shIWS1, shIWS1/WT-R and shIWS1/MT-R NCI-H522, and NCI-H1299 cells, by a lentiviral construct of wild-type HA-SETD2 (Supplementary Fig. 3d ). The failure to rescue the phenotype supports the model of SETD2 recruitment by phosphorylated IWS1. SETD2 is the only known H3K36 trimethyltransferase in mammalian cells [40] . However, histone methylation is a dynamic process [41] , and while SETD2 is the only H3K36 trimethyltransferase, there are several lysine methyltransferases, which catalyze mono- or dimethylation of histone H3 at K36 and may influence the SETD2 output. Transfection of the NCI-H522 and NCI-H1299 cells with siRNAs targeting a set of methyltransferases that are known to catalyze histone H3K36 mono- and dimethylation (NSD1, NSD2, and NSD3), or only dimethylation (SMYD2 and ASHL1) [42] , [43] , [44] , [45] , [46] , [47] , revealed that none of them contributes to the regulation of the alternative splicing of the U2AF2 exon 2 (Supplementary Fig. 3e ). The histone H3K36me3 marks are erased by KDM4A and KDM4C, two members of the KDM4 JmjC domain–histone demethylase family [48] , [49] , [50] . Ectopic expression of KDM4A, KDM4B, and KDM4C from lentivirus constructs in NCI-H522 and NCI-H1299 cells showed that none of the three altered the IWS1-dependent pattern of the U2AF2 alternative RNA splicing (Supplementary Fig. 3f ). This was expected for KDM4B, which does not target H3K36me3, and was used as a negative control, but it was unexpected for KDM4A and KDM4C. Overall, these data suggest that if KDM4A and KDM4C contribute to the demethylation of histone H3K36me3, they may do so, only under conditions that need to be determined. Alternatively, it is possible that the transcription-coupled SETD2-catalyzed histone H3K36 trimethylation may be erased by an oxygenase or demethylase, whose specificity toward histone H3K36me3 has not been determined yet. Recently, and after the completion of the ChIP experiments described above, we carried out ChIP-Seq experiments, addressing the binding of IWS1 and SETD2 and the distribution of H3K36me3 marks genome-wide in shIWS1/WT-R and shIWS1/MT-R, NCI-H522 cells. The unbiased data on the abundance of these markers in the U2AF2 gene were in general agreement with the ChIP data described above. Specifically, IWS1 was found to bind U2AF2 E2, independent of its phosphorylation, but SETD2 binding and H3K36me3 abundance on U2AF2 E2 increased only when IWS1 was phosphorylated (Fig. 3e ). The regulation of the alternative RNA splicing of the U2AF2 exon 2 by IWS1 phosphorylation, depends on the p52 isoform of the H3K36me3 reader LEDGF Our earlier studies had shown that the regulation of the FGFR2 alternative RNA splicing by IWS1 phosphorylation, depends on the reading of the histone H3K36me3 marks by MRG15 [22] . To determine whether MRG15 is also the reader of the IWS1-dependent alternative RNA splicing of U2AF2 , we knocked down MRG15 in both NCI-H522 and NCI-H1299 cells. Using RT-PCR and qRT-PCR to monitor the alternative RNA splicing of U2AF2 in these cells revealed that it is independent of MRG15 (Fig. 4a , left panels). In agreement with this result, the knockdown of the splicing repressor and binding partner of MRG15, PTB, also has no role on the RNA splicing of U2AF2 (Fig. 4a right panels), These results were in sharp contrast with the results of parallel control experiments, which confirmed that the knockdown of MRG15 or PTB in NCI-H522 and NCI-H1299 cells increases the FGFR2 IIIb/IIIc, transcript ratio, as expected (Supplementary Fig. 5a ) [11] , [22] . Given that in some cells, the knockdown of PTB upregulates PTBP2, which can compensate for the loss of PTB [51] , we also examined the expression of PTBP2 before and after the knockdown of PTB in these cells, and we observed no PTB-dependent changes (Fig. 4a , right upper panel). In addition, the knockdown of PTBP2, similar to the knockdown of PTB, did not affect the alternative RNA splicing of U2AF2 in either the NCI-H522 or NCI-H1299 cells (Supplementary Fig. 5b ), suggesting that U2AF2 mRNA splicing is also independent of PTBP2. Fig. 4: The regulation of the alternative splicing of the U2AF2 exon 2 by IWS1 and IWS1 phosphorylation, depends on the p52 isoform of the H3K36me3 reader LEDGF and its splicing partner SRSF1. a (Upper panel) Lysates of the indicated cells were probed with antibodies, as shown. RT-PCR addressing exon 2 U2AF2 splicing in the same cells. (Middle and Lower Panels) U2AF2 E2/E3 ±SD, was determined by quantification of the RT-PCR results and by qRT-PCR. b (Upper Panel) Lysates of NCI-H522 cells transfected with the indicated siRNAs, probed with antibodies, as shown. RT-PCR addressing exon 2 U2AF2 splicing. (Middle and Lower Panels) U2AF2 E2/E3 ±SD, was determined by quantification of the RT-PCR results and by qRT-PCR. c (Upper panel) Domains of the p52 and p75 LEDGF isoforms (see Ferris et al., 2010 50 ). (Middle panel) Western blot of the indicated NCI-H522 cells, probed for LEDGF expression and RT-PCR, addressing U2AF2 exon 2 splicing in the same cells. (Lower panels) U2AF2 E2/E3 ratio ±SD, was determined by quantification of the RT-PCR results and by qRT-PCR. d ChIP of p52/LEDGF in NCI-H522 cells, transduced with V5-p52/LEDGF. Mean fold enrichment in p52/LEDGF binding (anti-V5 IP, vs IgG control IP) to the indicated U2AF2 regions±SD. V5-p52/LEDGF expression, in figure S5G. e (Upper panel) Immunoblotting, showing SRSF1 expression in the indicated NCI-H522 cells. RT-PCR addressing U2AF2 exon 2 splicing. (Lower panels) U2AF2 E2/E3 ratio ±SD, was determined by quantification of the RT-PCR results and by qRT-PCR. f SRSF1 ChIP in the indicated V5-SRSF1-transduced NCI-H522 cells. Mean fold enrichment in SRSF1 binding (anti-V5 IP, vs IgG control IP) to the indicated U2AF2 regions±SD. V5-SRSF1 expression in Supplementary figure S6b. g RIP, addressing SRSF1 binding to U2AF2 RNA in panel f cells. Mean fold enrichment in SRSF1 binding (anti-V5 IP, vs IgG control IP) in the indicated U2AF2 regions ±SD. All assays were done, using three biological replicates, in triplicate. n.s non-significant, * p < 0.05, ** p < 0.01, *** p < 0.001, **** p < 0.0001 (one-sided unpaired t -test). h Phosphorylation of IWS1 recruits SETD2 in CTD of RNA Pol II. SetD2 trimethylates histone H3K36 co-transcriptionally. p52/LEDGF and its partner SRSF1, bind histone H3K36me3 promoting exon 2 inclusion in the mature U2AF2 transcript. Full size image To identify the H3K36me3 reader that may control the IWS1-dependent splicing of U2AF2 , we transfected NCI-H522 and NCI-H1299 cells with a control siRNA and siRNAs of the known H3K36me3 readers PHF1 [51] , BRPF1 [52] , MSH6 [53] , GLYR-1 [54] , and LEDGF [12] , [55] . Monitoring the effects of these transfections by RT-PCR and qRT-PCR revealed that only the knockdown of LEDGF phenocopied the knockdown of IWS1 on the alternative splicing of U2AF2 (Fig. 4b , Supplementary Fig. 5c ), suggesting that LEDGF is the sole H3K36me3 reader responsible for the U2AF2 alternative RNA splicing. To confirm this observation and to determine which isoform of LEDGF may be responsible for the detected phenotype, we used a lentiviral shRNA construct to knock down LEDGF, and we rescued the knockdown by transducing the cells with lentiviral constructs of the p75 and p52 isoforms of LEDGF (Fig. 4c , upper panel). Monitoring the effects of these transductions by RT-PCR and qRT-PCR revealed that only the p52 isoform rescues the U2AF2 alternative splicing phenotype. Importantly, the A51P mutant of the p52 isoform, which cannot bind histone H3K36me3 [56] , did not rescue the phenotype, suggesting that the rescue depends on the binding of p52 to the H3K36me3 marks (Fig. 4c , Supplementary Fig. 5d ). Notably, the knockdown of LEDGF did not affect the alternative RNA splicing of FGFR2 (Supplementary Fig. 5e ), suggesting that although H3K36me3 may be a common signal for the IWS1 phosphorylation-dependent RNA splicing of multiple targets, the RNA splicing regulators assembled by H3K36me3 on different targets are target-specific. If the p52 isoform of LEDGF regulates the alternative splicing of U2AF2 by reading the histone H3K36me3 marks, as suggested by the preceding data, and if the abundance of these marks depends on phosphorylated IWS1, the ectopic expression of p52/LEDGF should not rescue the shIWS1 and shIWS1/MT-R-induced alternative splicing phenotype. This was confirmed by experiments addressing the rescue of the U2AF2 RNA splicing in shControl, shIWS1, shIWS1/WT-R, and shIWS1/MT-R NCI-H522, and NCI-H1299 cells transduced with a lentiviral construct of wild-type V5-p52/LEDGF (Supplementary Fig. 5g ). The failure to rescue the phenotype supports the model of p52/LEDGF regulating the alternative RNA splicing of U2AF2 by reading the IWS1 phosphorylation and SETD2-dependent histone H3K36 trimethylation in the body of the U2AF2 gene. The preceding data provide strong genetic evidence that p52/LEDGF regulates the alternative RNA splicing of the U2AF2 by reading the IWS1 phosphorylation-dependent histone H3K36me3 marks. To confirm this interpretation of the results, we used ChIP to address the binding of p52/LEDGF on exons 2 and 3 of U2AF2 in shControl, shIWS1, shIWS1/WT-R and shIWS1/MT-R NCI-H522, and NCI-H1299 cells. The results confirmed that p52/LEDGF indeed binds U2AF2 exons 2 and 3 and that the binding depends on IWS1 phosphorylation and correlates with the abundance of histone H3K36me3 marks (Fig. 4d , Supplementary Fig. 5f ). We conclude that p52/LEDGF indeed regulates the alternative RNA splicing of U2AF2 , by reading the trimethylation of histone H3 at K36, downstream of IWS1 phosphorylation, and SETD2 recruitment to RNA Pol II. The p52 isoform of LEDGF regulates the alternative RNA splicing of U2AF2 , via its interaction with the RNA splicing factor SRSF1 It had been reported that the p52 isoform of LEDGF is transported to the nucleus, in response to signals targeting its unique CTD, and that in the nucleus it interacts with the splicing factor SRSF1 regulating the distribution of SRSF1 to alternatively spliced genes [12] . To investigate the role of SRSF1 in alternative RNA splicing, we knocked it down in NCI-H522 and NCI-H1299 cells and we showed that its loss reproduces the IWS1-knockdown phenotype of U2AF2 , but not FGFR2 alternative RNA splicing (Supplementary Fig. 6a ). The dependence of the U2AF2 exon 2 splicing on SRSF1, which was suggested by this result, was confirmed by rescue experiments with wild-type SRSF1 (Fig. 4e , Supplementary Fig. 6b ). We therefore conclude that SRSF1 regulates the alternative RNA splicing of the U2AF2 exon 2. However, SRSF1 did not rescue the U2AF2 splicing phenotype in shIWS1 and shIWS1/MT-R cells (Supplementary Fig. 6b ). This finding suggested that SRSF1 does not function independently, but instead provides a link between p52/LEDGF, recruited to IWS1 phosphorylation-dependent chromatin modification marks, and the RNA splicing machinery. To test this hypothesis, we transduced shControl, shIWS1, shIWS1/WT-R and shIWS1/MT-R NCI-H522, and NCI-H1299 cells with a V5-tagged SRSF1 lentiviral construct and we employed ChIP to address the binding of V5-SRSF1 to U2AF2 exons 2 and 3. U2AF2 TSS and GAPDH were again used as controls. The results confirmed the binding of SRSF1 to exons 2 and 3 only in shControl and shIWS1/WT-R cells (Fig. 4f and Supplementary Fig. 6c ), providing support to the proposed hypothesis. Based on the preceding data, we hypothesized that the binding to the chromatin-associated p52/LEDGF should bring SRSF1 into proximity with the nascent pre-mRNA, facilitating their interaction. Analysis of the U2AF2 mRNA sequence using the web-based pipeline RBP-map [57] , identified four potential SRSF1-binding sites (2 in U2AF2 exon 2, and 2 in exon 3) (Supplementary Fig. 6d ) [58] , providing additional support to this hypothesis. These findings raised the question whether SRSF1 binding could be common among genes undergoing IWS1 phosphorylation-dependent alternative RNA splicing, characterized by exon inclusion. To address this question, we analyzed the sequences of four alternatively spliced genes, which like U2AF2 , undergo IWS1 phosphorylation-dependent exon inclusion (Supplementary Fig. 1g–J ). This analysis identified SRSF1-binding motifs in the alternatively spliced and/or flanking exons in all these genes (Supplementary Fig. 6e–h ), and provided support to the hypothesis that SRSF1 binding may be a common feature of genes undergoing alternative RNA splicing via this mechanism. To experimentally address the proposed model, we carried out RNA-IP (RIP) experiments in the same shControl, shIWS1, and shIWS1/WT-R and shIWS1/MT-R NCI-H522 and NCI-H1299 cells, focusing on the binding of SRSF1 to the U2AF2 exon 2, intron 2, and exon 3. The results confirmed that SRSF1 binds primarily to exon 2, but only in the shControl and shIWS/WT-R cells (Fig. 4g , Supplementary Fig. 6i ), which parallels its binding to the H3K36me3-bound p52/LEDGF. We conclude that exon 2 inclusion in the U2AF2 mRNA in cells expressing wild-type IWS1 depends on the phosphorylation of IWS1 by AKT3, the recruitment of SETD2 to the CTD of RNA Pol II, the transcription-coupled histone H3K36 trimethylation, and the subsequent bridging of chromatin with the splicing machinery by LEDGF-p52 and SRSF1 (Fig. 4h ). U2AF65β, encoded by the exon 2-deficient splice variant of U2AF2 , does not interact with Prp19 The predominant splice variant of the U2AF2 mRNA in shIWS1 and shIWS1/MT-R cells is a variant, which lacks exon 2, the exon encoding the U2A65 N-terminal RS domain (Fig. 5a ). This domain is responsible for the interaction of U2AF65 with several factors that contribute to mRNA splicing and 3′ cleavage and polyadenylation [59] , [28] . One of these factors is Prp19, a component of the seven-member ubiquitin ligase complex Prp19C [32] , [33] , [34] , [35] . Fig. 5: IWS1 phosphorylation controls the CDCA5/ERK phosphorylation feedback loop, through U2AF2 alternative RNA splicing. a Functional domain composition of U2AF65. Numbers mark the domain boundaries. Exon 2 encodes the RS domain. b HEK-293T cells were transduced with the V5-tagged splice variants of U2AF2 , encoding V5-U2AF65α and V5-U2AF65β. Anti V5-U2AF65 immunoprecipitates and input lysates were probed with the indicated antibodies. c Anti-U2AF65, anti-IgG mouse isotype control immunoprecipitates and input lysates of NCI-H522 cells transduced with the indicated constructs were probed with antibodies, as shown. d (Upper panel) The ratio of spliced to unspliced CDCA5 and GUSB (control) RNAs was measured in the indicated NCI-H522 cells by qRT-PCR. (Middle and Lower panels) RIP assays of U2AF65 and Prp19 in the same cells. Anti-U2AF65 or anti-Prp19 IP, vs IgG control IP were used to calculate the mean fold binding enrichment in the indicated RNA regions ±SD. Primers listed in Supplementary Table 2. Primer location in Supplementary Fig. 7b . e (Upper panel) shIWS1 rescue by U2AF65α and U2AF65β. Spliced/unspliced RNA ratios of CDCA5 and GUSB, measured by qRT-PCR, as in Fig. 5d. (Middle and Lower panels) RIP assays of U2AF65 and Prp19 in the same cells. Data presented as in figure 5d. f Cytosolic CDCA5 mRNA levels in the indicated shIWS1-transduced cells were rescued by IWS1 and U2AF65α, as determined by q-RT-PCR. GAPDH- normalized CDCA5 mRNA ±SD. Validation of fractionation in Supplementary Fig. 7e . g Lysates of NCI-H522 cells, transduced with the indicated constructs, were probed with antibodies, as shown. DM-A and DM-E are the S79/S209AA and S79/S209EE Sororin mutants, respectively. h (Upper panels) Lysates of KRAS and EGFR mutant cell lines, transduced with the indicated constructs, were probed with antibodies as shown. RT-PCR, using U2AF2 exon 1 and 3 primers. (Lower Left panel) Bars show the qRT-PCR-determined U2AF2 E2/E3 ratios in NCI-H522 and NCI-H1299 cells, and in the KRAS and EGFR mutant cell lines, relative to the shControl±SD. (Lower Right panel) Bars show the shIWS1-induced percent reduction of ERK-phosphorylation in the same cell lines, normalized to tubulin ± SD. EGFR mutant and non-mutant cells were compared, using a one-way ANOVA. All assays were in triplicate, on three biological replicates. n.s non-significant, * p < 0.05, ** p < 0.01, *** p < 0.001, **** p < 0.0001 (one-sided unpaired t -test). Full size image Using co-immunoprecipitation in HEK-293T cells transduced with V5-tagged U2AF2 constructs containing or lacking exon 2, we confirmed that whereas the protein encoded by the exon 2-containing splice variant (U2AF65α) interacts with endogenous Prp19, the protein encoded by the exon 2-deficient splice variant (U2AF65β), does not (Fig. 5b ). More important, co-immunoprecipitation of endogenous U2AF65 from shControl, shIWS1, shIWS1/WT-R, and shIWS1-MT-R NCI-H522 and NCI-H1299 cells, revealed that the two proteins co-immunoprecipitate only in shControl and shIWS1-WT-R cells, which express primarily U2AF65α (Fig. 5c , Supplementary Fig. 7a ). These data confirmed that the interaction of U2AF65 with Prp19 depends on the sequence encoded by U2AF2 exon 2, whose inclusion in the transcript is regulated by IWS1 phosphorylation. The splicing of the U2AF2 mRNA, downstream of IWS1 phosphorylation, regulates the mRNA splicing of CDCA5 and the abundance of its protein product Sororin It had been previously shown that U2AF65 binds RNA Pol II and recruits Prp19 to the newly synthetized pre-mRNA, promoting co-transcriptional RNA splicing [60] . One of the genes whose RNA splicing depends on the U2AF65-dependent recruitment of Prp19 to RNA Pol II, is CDCA5 , the gene encoding Sororin, a component of the cohesin complex [36] . Given that U2AF65β, which is the predominant U2AF65 isoform expressed in shIWS1 and shIWS1/MT-R cells does not bind Prp19, we hypothesized that the RNA splicing of CDCA5 in these cells will be impaired. To address this hypothesis, we employed qRT-PCR to determine the ratio of spliced and unspliced CDCA5 RNA in shControl, shIWS1, shIWS1/WT-R, and shIWS1/MT-R NCI-H522 and NCI-H1299 cells. The RNA splicing of GUSB , does not depend on the U2AF65 interaction with Prp19 [36] , and it was used as the negative control. The results confirmed that whereas the RNA splicing of CDCA5 is impaired in both the shIWS1 and shIWS1/MT-R cells, the RNA splicing of GUSB is not (Fig. 5d , Supplementary Fig. 7b and c , upper panels). More important, the splicing defect was rescued by U2AF65α but not by U2AF65β (Fig. 5e , Supplementary Fig. 7d , upper panels). To determine how IWS1 phosphorylation regulates CDCA5 RNA splicing, we performed RNA immunoprecipitation (RIP) experiments in shControl, shIWS1, shIWS1/WT-R, and shIWS1/MT-R NCI-H522 and NCI-H1299 cells. The results confirmed that the two splice variants of U2AF65 bind equally well the CDCA5 pre-mRNA, as well as the control GUSB pre-mRNA, as expected (Fig. 5d, e , Supplementary Fig. 7c and Supplementary Fig. 7d , middle panels). However, the binding of Prp19 to the same pre-mRNA regions of CDCA5 was significantly impaired in shIWS1 and shIWS1/MT-R cells, which predominantly express the U2AF65β isoform (Fig. 5d , Supplementary Fig. 7c , lower panels). More important, the impaired Prp19 binding to the pre-mRNA of CDCA5 in shIWS1-transduced cells, was rescued by U2AF65α, but not U2AF65β (Fig. 5e and Supplementary Fig. 7d , lower panels). Given that only spliced mRNAs are transported out of the nucleus, we used qRT-PCR to determine the abundance of cytosolic CDCA5 mRNA in shControl, shIWS1, shIWS1/WT-R, and shIWS1/MT-R and shIWS1 NCI-H522 and NCI-H1299 cells, as well as in shIWS1 cells, before and after rescue with U2AF65α or U2AF65β. To this end, we fractionated the cells into nuclear and cytosolic compartments and we probed western blots of the fractions with antibodies to Lamin A/C and GAPDH, to confirm the fractionation (Supplementary Fig. 7e ). The results confirmed that the mature CDCA5 mRNA was present at low abundance in the cytoplasmic fraction of shIWS1 and shIWS1/MT-R cells as expected and that its abundance was restored in shIWS1 cells rescued with U2AF65α, but not U2AF65β (Fig. 5f ). To determine whether the CDCA5 RNA splicing defect in shIWS1 and shIWS1/MT-R NCI-H522 and NCI-H1299 cells prevents the expression of its protein product Sororin, we examined the expression of Sororin in these cells, along with the expression of IWS1, pIWS1, U2AF65, and Prp19 by western blotting. The results confirmed that the expression of Sororin was indeed impaired as expected, in shIWS1 and shIWS1/MT-R NCI-H522 and NCI-H1299 cells. More important, the expression of Sororin was again rescued by U2AF65α, but not by U2AF65β (Fig. 5g , Supplementary Fig 7f , upper panels). Sororin and p-ERK form a positive feedback loop, which is activated by IWS1 phosphorylation and promotes the expression of CDK1 and Cyclin B1 It had been shown previously that the downregulation of Sororin leads to reduced ERK phosphorylation at Y202/T204 in human colorectal cancer (CRC) and human hepatocellular carcinomas (HCC) [61] , [62] . Assuming that the link between Sororin abundance and ERK phosphorylation is conserved in lung adenocarcinomas, these findings suggested that the knockdown of IWS1 and its replacement by the phosphorylation-site mutant IWS1S720A/T721A in NCI-H522 and NCI-H1299 cells would also result in inhibition of ERK phosphorylation. This question was addressed and the results confirmed the prediction. More important, the reduction of p-ERK in shIWS1 cells was rescued by U2AF65α, but not by U2AF65β (Fig. 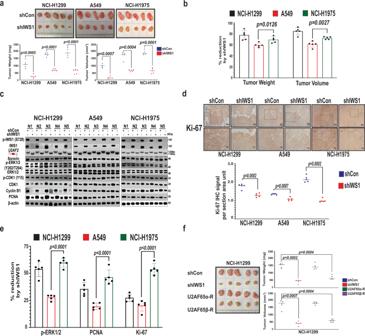Fig. 7: IWS1 phosphorylation controls tumour growth in vivo, by regulating the U2AF2/Sororin/ERK axis. a(Upper panels) NSG mice were injected subcutaneously with shControl or shIWS1 NCI-H1299, A549, or NCI-H1975 cells. (N= 5 mice/group). Images of tumors, harvested at 4 weeks (NCI-H1299, NCI-H1975) or 6 weeks (A549) from the time of inoculation. (Lower panels) Scatter plots showing the weight and volume of individual tumors. The horizontal lines indicate mean tumor weight or volume. Statistical analyses were done using the one-sided pairedt-test.bshIWS1-induced percent reduction of tumor weight and tumor volume, calculated from the weight and volume of the tumors induced by shIWS1 and shControl cells in panela. Bars show the mean percent reduction±SD. Statistical analyses were done using the one-sided unpaired t-test.cCell lysates derived from NCI-H1299, A549 and NCI-H1975 (shControl and shIWS1) mouse xenografts, were probed with the indicated antibodies. RT-PCR on RNA from the same cells, using primers forU2AF2exons 1 and 3.d(Upper panels) The indicated shControl and shIWS1, formalin-fixed, paraffin-embedded tumor samples were stained with the Ki-67 antibody. Boxes in the upper images delineate the area of higher magnification shown in the lower images. Scale bar in the right lower corner of each image. (Lower panels) Scatter plots show the Ki-67 IHC signal per section area unit in shControl and shIWS1 tumors. The horizontal lines show mean Ki-67 signals. Statistical analyses were performed, using the one-sided pairedt-test.eShIWS1-induced percent reduction of the phosphor-ERK, PCNA and Ki-67 signals in the xenograft tumors. Bars show the mean signal reduction, based on quantification of the Western blot data in panelc(p-ERK and PCNA) and IHC data in figure 7e (Ki-67) ± SD. Statistics were performed using the one-sided unpairedt-test.f(Left panels) shControl, and shIWS1 NCI-H1299 cells, as well as shIWS1 NCI-H1299 cells rescued with U2AF65α, or U2AF65β, were injected subcutaneously in NSG mice, as in the experiment in panela(N= 5 mice/group). Images of tumors harvested at 4 weeks from the time of inoculation. (Right panels) Scatter plots showing the weight and volume of the harvested tumors. The horizontal lines indicate mean tumor weight or volume. Statistical analyses were performed with the one-sided pairedt-test. 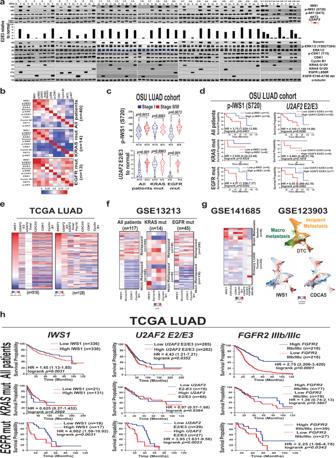Fig. 8: The p-IWS1/U2AF2 pathway is active in human lung adenocarcinomas and impacts tumour grade, stage, metastatic potential and treatment relapse in patients withEGFRmutant, but notKRASmutant tumors. aLysates of 30 LUAD samples paired with NAT, and 10 unpaired samples, were probed with the indicated antibodies. RT-PCR ofU2AF2in the same samples was performed, using exon 1 and 3 primers. Bars show theU2AF2E2/E3 exon ratio in the tumors in the upper panel, relative to the average of the 30 normal samples.bCorrelation heatmaps between components of the IWS1 phosphorylation pathway, in the LUADs in a. Correlation coefficients were calculated using simple linear regression. The values and the statistical confidence of all the comparisons can be found in Supplementary Table 5.cViolin plots showing the abundance of IWS1 phosphorylation and theU2AF2E2/E3 ratio (right) in stage I and Stage II/III tumors. Data shown for all tumors in panelsaandb, and selectively forEGFRorKRASmutant tumors. The horizontal black lines indicate mean values for phospho-IWS1 levels andU2AF2E2/E3 ratios. Statistical analyses were performed using the one-sided unpairedt-test.dKaplan-Meier Curves of phosphor-IWS1 andU2AF2E2/E3 ratios in the LUAD cohort in panela. Statistical analyses were performed using the one-sided log rank test and Cox’s proportional hazards model.eHeat Maps showing the correlation of IWS1 or SRSF1 with components of the IWS1/U2AF2 pathway in the TCGA LUAD database using log2normalized counts.fHeatmaps showing the expression of IWS1 pathway components in the tumors of the GSE13213 dataset.g(Left panel) Heat Maps showing expression of IWS1 pathway components in resected brain metastases and primary lung adenocarcinomas. RNA-seq data for metastatic lesions were derived from the GSE141685 dataset and for primary LUADs from TCGA. (Right upper panel) scRNA-Seq data from GSE123903. Force-directed layout/t-SNE of all metastatic tumor cells isolated from patient-derived mouse xenografts (Laughney et al., 202071), colored by source, (Right lower panel) Force-directed layout (as in the upper panel) of all xenograft tumor cells colored forz-normalizedIWS1andCDCA5expression.hKaplan–Meier curves showing the impact of IWS1,U2AF2E2/E3 andFGFR2IIIb/IIIc ratios on patient survival in the indicated patients in the TCGA LUAD database. Statistical analyses were performed as in paneld. 5g , Supplementary Fig. 7f , lower panels), confirming that the activity of the p-IWS1/Sororin/p-ERK axis in lung adenocarcinomas depends on the alternative RNA splicing of U2AF2 . Sororin is phosphorylated by ERK at Ser79 and Ser209 [63] . This observation raised the question whether it is Sororin, or the phosphorylated Sororin, which promotes the phosphorylation of ERK. Experiments addressing this question showed that whereas wild-type Sororin and the Sororin phosphomimetic mutant S79E/T209E (Sororin DM-E) rescue the phosphorylation of ERK in shIWS1 cells, the S79A/S209A (Sororin DM-A) mutant does not (Fig. 5g , Supplementary Fig. 7f , lower panels). We conclude that ERK phosphorylation is promoted by phosphorylated Sororin, and that Sororin and ERK are components of a positive feedback loop, which is controlled by AKT-dependent IWS1 phosphorylation and U2AF2 alternative RNA splicing and is active in lung adenocarcinomas. Inhibiting the expression of Sororin results in downregulation of CDK1 and Cyclin B1 [61] , [62] . This observation suggested that IWS1 phosphorylation, which regulates the abundance of Sororin, may also regulate the expression of CDK1 and Cyclin B1. Experiments addressing this hypothesis showed that shIWS1 and shIWS1/MT-R NCI-H522 and NCI-H1299 cells indeed express reduced levels of CDK1, phosphor-CDK1(Y15), and Cyclin B1, and that the downregulation of these molecules in shIWS1 cells is rescued by wild-type Sororin and Sororin DM-E, but not Sororin DM-A (Fig. 5g , Supplementary Fig. 7f , lower panels). Based on these data, we conclude that the regulation of CDK1 and Cyclin B1 by IWS1 phosphorylation depends on the activation of the Sororin-ERK phosphorylation feedback loop. The IWS1 phosphorylation-dependent alternative RNA splicing of U2AF2 regulates ERK phosphorylation in lung adenocarcinoma cell lines, including those harboring EGFR or KRAS mutations EGFR and KRAS are frequently mutated in human lung adenocarcinomas and the mutated forms of these genes promote oncogenesis by activating multiple signaling pathways, including the ERK pathway [64] , [65] . Given that IWS1 phosphorylation also promotes the activation of ERK via the Sororin/p-ERK positive feedback loop, we asked whether IWS1 phosphorylation influences ERK phosphorylation in lung adenocarcinoma cell lines, harboring KRAS (A549 and NCI-H460) or EGFR (NCI-H1975, PC-9, and NCI-H1650) mutations. The results showed that IWS1 phosphorylation and U2AF2 exon 2 inclusion were independent of the EGFR or KRAS mutational status (Fig. 5h ). In addition, Sororin expression and ERK phosphorylation were reduced in all shIWS1 and shIWS1/MT-R cell lines, including those with KRAS or EGFR mutations (Fig. 5h ). We conclude that the Sororin/p-ERK positive feedback loop defines a pathway of ERK regulation, which has the potential to modulate ERK activation by KRAS or tyrosine kinase receptor signals. Surprisingly, the role of this pathway in the regulation of EGFR -induced ERK activation signals was more robust than its role in the regulation of KRAS -induced signals (Fig. 5h ). The AKT/IWS1/ U2AF2 pathway promotes cell proliferation by activating the Sororin/ERK positive feedback loop Our earlier studies had shown that IWS1 phosphorylation promotes the proliferation of the lung adenocarcinoma cell lines NCI-H522 and NCI-H1299 [22] . Given that the Sororin/ERK positive feedback loop, downstream of the IWS1-dependent inclusion of exon 2 in the U2AF2 mRNA, upregulates CDK1 and Cyclin B1, we hypothesized that IWS1 promotes cell proliferation, by activating this loop. To address this hypothesis, we examined the rate of proliferation of shControl, shIWS1, shIWS1/Sororin WT, shIWS1/Sororin DM-A, and shIWS1/Sororin DM-E NCI H522 and NCI-H1299 cells growing under standard culture conditions. The results showed that cell proliferation was inhibited by shIWS1 and that the inhibition was rescued by wild-type Sororin and Sororin DM-E but not by Sororin DM-A. Importantly, they also showed that the phosphomimetic Sororin mutant (DM-E) promotes cell proliferation more robustly than the wild-type protein. In addition, the experiment in Fig. 6b shows that whereas the shIWS1-induced proliferation defect in NCI-H522 and NCI-H1299 cells is rescued by U2AF65α, it is not rescued by U2AF65β, confirming the role of U2AF2 alternative RNA splicing in this pathway. Fig. 6: IWS1 phosphorylation promotes cell proliferation by controlling a Sororin/ERK phosphorylation feedback loop, through U2AF2 RNA splicing. a , b Growth curves of shControl and shIWS1 NCI-H522 and NCI-H1299 cells, growing in fully supplemented media, before and after rescue with Sororin (wt or mutants), or U2AF65α/U2AF65β. Experiment was done in triplicate and proliferation was expressed as mean percent confluence ±SD. P values (one-sided unpaired t -test) were calculated for the endpoint measurements. * p < 0.05, ** p < 0.01, *** p < 0.001, **** p < 0.0001. b Growth curves of shControl and shIWS1 A549 and NCI-H1975 cells. c Growth curves of the same shIWS1 cells rescued with U2AF65α or U2AF65β. Proliferation in panels c and d was measured as in panels a and b . d (Upper panel) Cell cycle profiles of the indicated propidium iodide (PI)-stained cell lines. One representative, out of three biological replicates. Mean percentages of cells in different cell cycle phases in red. (Lower panel) shIWS1-induced percent change of cells in G2/M±SD. Statistical analysis was performed using a one-sided unpaired t -test, * p < 0.05. Gating strategy in supplementary figure 8a. e NCI-H1299 cells were sorted into G0/G1, S and G2/M fractions. Lysates of sorted cells were probed with the indicated antibodies. RT-PCR on RNA from the same cells, using primers for U2AF2 exons 1 and 3. Gating strategy in supplementary figure 8a. f qRT-PCR-determined expression of IWS1 , CDCA5 and U2AF2 , relative to GAPDH±SD. SD was calculated based on three biological replicates. g ChIC-determined mean fold enrichment of IWS1, SETD2 and H3K36me3 in cell cycle fractionated cells in the indicated regions of the U2AF2 RNA±SD. h qRT-PCR-based calculation of the mean U2AF2 E2/E3 ratio in S and G2/M, relative to G0/G1 cells ±SD. SD was calculated based on three biological replicates * p < 0.05, ** p < 0.01, *** p < 0.001, **** p < 0.0001. (one-sided unpaired t -test). i IWS1 expression is induced during the S and G2/M phases of the cell cycle. Following phosphorylation by AKT3, IWS1 orchestrates the cell cycle-dependent assembly of epigenetic complexes on the U2AF2 gene. This promotes the inclusion of exon 2 in the U2AF2 mRNA. U2AF65α, encoded by the exon 2-containing U2AF2 mRNA, interacts with Prp19, promoting CDCA5 splicing and the expression of Sororin. The latter is phosphorylated by ERK, and promotes ERK phosphorylation, in a positive feedback loop, which stimulates proliferation of lung adenocarcinomas. Full size image Additional experiments showed that IWS1 also promotes the proliferation of A549 and NCI-H1975 cells and that its role in the proliferation of NCI-H1955 cells, which harbor an activating EGFR mutation, is significantly more robust than its role in the proliferation of A549 cells, which harbor a KRAS mutation (Fig. 6c , Supplementary Fig. 9a ). Although it is difficult to determine the significance of an observation that is based on only two cell lines, we wish to point out that this observation is in agreement with the results of the experiment in Fig. 5h , which shows that IWS1 phosphorylation activates the Sororin/ERK positive feedback loop more strongly in EGFR mutant than in KRAS mutant cell lines. Importantly, the observed antiproliferative effect of the knockdown of IWS1 in these cell lines, also depends on the alternative RNA splicing of U2AF2 , as determined by the phenotypic rescue of shIWS1, by U2AF65α, but not by U2AF65β (Fig. 6d ). The role of U2AF2 alternative RNA splicing in the regulation of cell proliferation by IWS1 in all four cell lines was also supported by the results of immunoblotting experiments addressing the expression of the proliferation marker PCNA, which showed that shIWS1 reduces the expression of PCNA, and that the reduced PCNA expression can be rescued again by U2AF65α, but not U2AF65β (Supplementary Fig. 9b ). The activation of the Sororin/p-ERK positive feedback loop and the induction of its downstream targets CDK1 and Cyclin B1 by IWS1 phosphorylation, suggested that IWS1 promotes cell proliferation by facilitating progression through the G2/M phase of the cell cycle. To address this hypothesis, we stained log-phase cultures of shControl, shIWS1, shIWS1/U2AF65α, and shIWS1/U2AF65β-rescued NCI-H522, NCI-H1299, A549, and NCI-H1975 cells with propidium iodide and we analyzed them by flow cytometry. The results of this experiment confirmed the hypothesis by showing that the shIWS1 cells accumulate in G2/M, and that the G2/M arrest is rescued by U2AF65α, but not by U2AF65β (Fig. 6e ). In agreement with the results of the experiments in Figs. 5 h and 6c , the shIWS1-induced percent reduction of cell proliferation (Supplementary Fig. 9a ) and the percent increase of cells in G2/M (Fig. 6e , lower panel) were more robust in the EGFR mutant (NCI-H1975) than in the KRAS mutant (A549) cell line. Given the small number of cell lines, these experiments provide only an indication that the regulation of cell proliferation by IWS1 may be more robust in lung adenocarcinomas with EGFR mutations. Strong support to this hypothesis was provided by experiments in primary lung adenocarcinomas, which will be presented in subsequent sections. IWS1 expression and phosphorylation, and U2AF2 alternative RNA splicing, fluctuate during progression through the cell cycle The preceding findings suggest that an RNA splicing event, regulated by the AKT-mediated phosphorylation of IWS1, plays a critical role in cell cycle progression. It is known that the expression or activity of molecules critically involved in the regulation of the cell cycle, tend to fluctuate as the cells transit from one phase of the cell cycle to the next [66] . We therefore examined the expression and phosphorylation of IWS1, the pattern of U2AF2 alternative RNA splicing, and the expression of Sororin, along with the expression of SETD2 and the abundance of H3K36me3 chromatin marks, in NCI-H1299 cells, sorted into G1, S, and G2/M pools. To separate cells in different phases of the cell cycle into distinct pools, we stained exponentially growing cells with a carboxyfluorescein succinimidyl ester (CFSE)-like DNA dye, and we sorted them by FACS [67] (Supplementary Fig. 8 ). The cell cycle markers we used to validate the sorting, were Cyclin E1 (G1 phase), CDC25A (S phase), and phosphorylated Histone H3 (S10) (G2/M phase). Western blotting of cells in different pools revealed that IWS1, phospho-IWS1, Sororin, SETD2, and histone H3K36me3 are indeed upregulated in S and G2/M (Fig. 6f ). Whereas IWS1 expression and phosphorylation were upregulated most abundantly during S phase, the upregulation of Sororin, SETD2, and Histone H3K36me3 was more robust during G2/M (Fig. 6f ), as previously reported [36] , [68] . RT-PCR, using RNA derived from the same cells, revealed that the inclusion of exon 2 in the U2AF2 mRNA, also fluctuates with the cell cycle, and parallels the expression and phosphorylation of IWS1 (Fig. 6f ). qRT-PCR, monitoring the expression of IWS1 and CDCA5 , revealed that the abundance of the RNA transcripts of these genes (Fig. 6g ) parallels the abundance of their protein products (Fig. 6f ), which indicates that the fluctuation of their expression during the cell cycle is regulated at the RNA level. Parallel qRT-PCR experiments revealed that although the pattern of U2AF2 mRNA splicing changes as the cells progresses through the cell cycle, the overall abundance of the U2AF2 RNA does not change (Fig. 6g ). Chromatin immunocleavage (ChIC) experiments revealed increased binding of IWS1 on U2AF2 exons 2 and 3 during S and G2/M, with highest binding during S phase (Fig. 6h ). Finally, although SETD2 and H3K36me3 are more abundant during G2/M (Fig. 6f ), the binding of SETD2, the abundance of H3K36me3 chromatin marks, and the U2AF2 E2/E3 ratio parallel the abundance of IWS1 and its binding to the U2AF2 gene, which are the highest during S phase (Fig. 6h , i). The cell cycle regulation of the pathway and the potential mechanisms involved are outlined in Supplementary Fig. 9c . Overall, these data provide strong support for the model in Fig. 6j . IWS1 expression and AKT activation increase as the cells enter S phase and their increase is maintained during G2M. AKT (primarily AKT3) phosphorylates IWS1 at S720/T721. The IWS1 phosphorylation signals the recruitment of SETD2 to the CTD of RNA Pol II and promotes the trimethylation of histone H3 at K36 in U2AF2 and other target genes. In the case of U2AF2 , H3K36me3 is recognized by p52/LEDGF, which interacts with the RNA splicing regulator SRSF1, and promotes the inclusion of exon 2 in the mature U2AF2 mRNA transcript. The exon 2-containing U2AF2 transcript encodes U2AF65α, while the exon 2-deficient transcript encodes U2AF65β. Of those, only U2AF65α, whose expression is promoted by IWS1 phosphorylation, binds Prp19 and facilitates the proper splicing of CDCA5 , leading to accumulation of its protein product Sororin, during S and G2/M. Finally, Sororin and ERK form a positive feedback loop, with ERK phosphorylating Sororin and Sororin promoting indirectly the phosphorylation of ERK. Activation of this loop plays an important role in the maintenance of ERK phosphorylation, and in the progression through the G2/M phase of the cell cycle. The AKT/IWS1/U2AF2/CDCA5/ERK pathway transforms hTert-immortalized human bronchial epithelial cells (hTert-HBEC) in culture The role of the AKT/IWS1/ U2AF2 /CDCA5/ERK pathway in cell cycle regulation raised the question whether this pathway also transforms cells in culture. To address this question, we used a soft agar-based assay to determine whether activation of the pathway promotes anchorage-independent growth of hTert-HBEC cells. The cells were first transduced with lentiviral constructs of constitutively active AKT3 (MyrAKT3 and AKT3-DD), the phosphomimetic IWS1-DE mutant, U2AF65α, and U2AF65β, encoded by the two splice variants of U2AF2 and Sororin, wild type, and its phosphomimetic and phosphorylation-deficient mutants (DM-E and DM-A, respectively). The expression of the proteins encoded by all the transduced constructs was determined by western blotting (Supplementary Fig. 10a ). Cells were plated in triplicate and they were imaged seven days later, using an incucyte live-cell imager (Supplementary Fig. 10b ). Live-cell numbers were measured immediately after imaging, as described in the experimental procedures and the data are presented as the mean number ± SD of three independent cultures (Supplementary Fig. 10c ). The results of this experiment fully support the role of this pathway in cell transformation, by showing that whereas constitutively active AKT3, wild-type Sororin, the phosphomimetic mutants of IWS1, Sororin (IWS1 DE and Sororin DM-E), and U2AF65α transform cells in culture, the phosphorylation-deficient mutant of Sororin (Sororin DM-A) and U2AF65β does not. The AKT/IWS1/U2AF2/CDCA5/ERK pathway controls tumor growth in vivo Our earlier studies had shown that the loss of IWS1, or IWS1 phosphorylation, inhibits tumor growth in a mouse xenograft model [22] . To confirm this observation, we repeated the experiment in two lung adenocarcinoma cell lines not tested before (A549 and NCI-H1975), and in NCI-H1299 cells, which were used as the positive control. Cells transduced with shIWS1 or shControl constructs, were inoculated subcutaneously, in the flanks of immunocompromised NSG mice. Mice injected with NCI-H1299 and NCI-H1975 cells were sacrificed at 4 weeks post injection, while mice injected with A549 cells were sacrificed at 6 weeks post-injection. The results revealed that the IWS1 knockdown reduced tumor growth and that the growth reduction was least pronounced in tumors derived from the KRAS mutant cell line A549 (Fig. 7a , b). The weak growth reduction of tumors derived from shIWS1 A549 cells paralleled the weak inhibition of ERK phosphorylation (Fig. 5h ) and cell proliferation (Supplementary Fig. 9a ) induced by the knockdown of IWS1 in these cells. Fig. 7: IWS1 phosphorylation controls tumour growth in vivo, by regulating the U2AF2/Sororin/ERK axis. a (Upper panels) NSG mice were injected subcutaneously with shControl or shIWS1 NCI-H1299, A549, or NCI-H1975 cells. ( N = 5 mice/group). Images of tumors, harvested at 4 weeks (NCI-H1299, NCI-H1975) or 6 weeks (A549) from the time of inoculation. (Lower panels) Scatter plots showing the weight and volume of individual tumors. The horizontal lines indicate mean tumor weight or volume. Statistical analyses were done using the one-sided paired t -test. b shIWS1-induced percent reduction of tumor weight and tumor volume, calculated from the weight and volume of the tumors induced by shIWS1 and shControl cells in panel a . Bars show the mean percent reduction±SD. Statistical analyses were done using the one-sided unpaired t-test. c Cell lysates derived from NCI-H1299, A549 and NCI-H1975 (shControl and shIWS1) mouse xenografts, were probed with the indicated antibodies. RT-PCR on RNA from the same cells, using primers for U2AF2 exons 1 and 3. d (Upper panels) The indicated shControl and shIWS1, formalin-fixed, paraffin-embedded tumor samples were stained with the Ki-67 antibody. Boxes in the upper images delineate the area of higher magnification shown in the lower images. Scale bar in the right lower corner of each image. (Lower panels) Scatter plots show the Ki-67 IHC signal per section area unit in shControl and shIWS1 tumors. The horizontal lines show mean Ki-67 signals. Statistical analyses were performed, using the one-sided paired t -test. e ShIWS1-induced percent reduction of the phosphor-ERK, PCNA and Ki-67 signals in the xenograft tumors. Bars show the mean signal reduction, based on quantification of the Western blot data in panel c (p-ERK and PCNA) and IHC data in figure 7e (Ki-67) ± SD. Statistics were performed using the one-sided unpaired t -test. f (Left panels) shControl, and shIWS1 NCI-H1299 cells, as well as shIWS1 NCI-H1299 cells rescued with U2AF65α, or U2AF65β, were injected subcutaneously in NSG mice, as in the experiment in panel a ( N = 5 mice/group). Images of tumors harvested at 4 weeks from the time of inoculation. (Right panels) Scatter plots showing the weight and volume of the harvested tumors. The horizontal lines indicate mean tumor weight or volume. Statistical analyses were performed with the one-sided paired t -test. Full size image To address the mechanism of the inhibition of tumor growth by shIWS1, we first confirmed the efficiency of the IWS1 knockdown, by probing western blots of tumor cell lysates with anti-IWS1 and anti-phospho-IWS1 (S720) antibodies (Fig. 7c ). Following this, we employed RT-PCR and qRT-PCR to address the usage of exon 2 in the U2AF2 mRNA in the tumors. The results confirmed that the knockdown of IWS1 has no effect on the total U2AF2 mRNA levels (Supplementary Fig. 11a , upper panel), but promotes the exclusion of exon 2 from U2AF2 mRNA (Fig. 7c , Supplementary Fig. 11a , lower panel). Probing both tumor lysates and tissue sections with antibodies to regulators and targets of the Sororin/ERK feedback loop, confirmed that its activity was reduced in tumors derived from shIWS1 cells (Fig. 7c , Supplementary Fig. 11b ). Measuring the abundance of the proliferation markers PCNA (western blotting) and Ki-67 (immunohistochemistry), confirmed that the expression of these markers was also reduced in the shIWS1 xenografts (Fig. 7c , d). Quantitative analyses of the western blot (p-ERK and PCNA) and IHC data (Ki-67) showed more robust downregulation of all these markers in tumors derived from the shIWS1-transduced NCI-H1975 than A549 cells (Fig. 7e ), as expected. To determine whether the regulation of xenograft growth by phosphorylated IWS1 depends on the inclusion of exon 2 in the U2AF2 mRNA, we knocked down IWS1 in NCI-H1299 cells and we rescued the knockdown with U2AF65α or U2AF65β (U2AF65α-R and U2AF65β-R). These cells, as well as shControl and shIWS1 NCI-H1299 cells, were injected in the flanks of NSG mice, as described in the “Methods” section. The results of this experiment (Supplementary Fig. 11c and Fig. 7f ) confirmed that the U2AF2 alternative RNA splicing plays a critical role in the regulation of tumor growth by phosphorylated IWS1. The xenograft data presented here were in full agreement with the data on the role of the IWS1 phosphorylation pathway in cell proliferation (Fig. 6a , b) and cell transformation in culture (Supplementary Fig. 10 ). The AKT/IWS1/U2AF2/CDCA5/ERK pathway is active in human lung adenocarcinomas and impacts tumor grade, stage, metastatic potential, and treatment relapse in patients with EGFR mutant, but not KRAS mutant tumors To determine whether the pathway activated by IWS1 phosphorylation and leading to Sororin expression and ERK phosphorylation is active in human lung adenocarcinomas (LUAD), we examined the expression and phosphorylation of IWS1, the alternative splicing of U2AF2 , and the abundance of ERK and phosphor-ERK, CDK1, and phosphor-CDK1 and cyclin B1 in a set of 40 human LUAD samples. For 30 of these tumors, normal adjacent tissue (NAT) was also available and was tested on parallel with the matching tumor sample. The results showed that the expression and phosphorylation of IWS1, the E2/E3 ratio in the U2AF2 mRNA, and the expression and/or phosphorylation of downstream targets of the pathway, were all higher in the tumors, than in normal tissues (Fig. 8a ). Importantly, IWS1 phosphorylation promoted the inclusion of exon 2 in the U2AF2 mRNA, but it did not alter the expression of U2AF2 (Supplementary Fig. 12a ). Overall, these data confirmed that the pathway is active in the tumors, but not in NAT. Fig. 8: The p-IWS1/U2AF2 pathway is active in human lung adenocarcinomas and impacts tumour grade, stage, metastatic potential and treatment relapse in patients with EGFR mutant, but not KRAS mutant tumors. a Lysates of 30 LUAD samples paired with NAT, and 10 unpaired samples, were probed with the indicated antibodies. RT-PCR of U2AF2 in the same samples was performed, using exon 1 and 3 primers. Bars show the U2AF2 E2/E3 exon ratio in the tumors in the upper panel, relative to the average of the 30 normal samples. b Correlation heatmaps between components of the IWS1 phosphorylation pathway, in the LUADs in a. Correlation coefficients were calculated using simple linear regression. The values and the statistical confidence of all the comparisons can be found in Supplementary Table 5. c Violin plots showing the abundance of IWS1 phosphorylation and the U2AF2 E2/E3 ratio (right) in stage I and Stage II/III tumors. 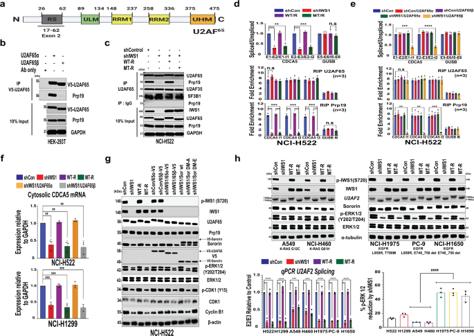Data shown for all tumors in panels a and b , and selectively for EGFR or KRAS mutant tumors. The horizontal black lines indicate mean values for phospho-IWS1 levels and U2AF2 E2/E3 ratios. Fig. 5: IWS1 phosphorylation controls the CDCA5/ERK phosphorylation feedback loop, through U2AF2 alternative RNA splicing. aFunctional domain composition of U2AF65. Numbers mark the domain boundaries. Exon 2 encodes the RS domain.bHEK-293T cells were transduced with the V5-tagged splice variants ofU2AF2, encoding V5-U2AF65α and V5-U2AF65β. Anti V5-U2AF65 immunoprecipitates and input lysates were probed with the indicated antibodies.cAnti-U2AF65, anti-IgG mouse isotype control immunoprecipitates and input lysates of NCI-H522 cells transduced with the indicated constructs were probed with antibodies, as shown.d(Upper panel) The ratio of spliced to unsplicedCDCA5and GUSB (control) RNAs was measured in the indicated NCI-H522 cells by qRT-PCR. (Middle and Lower panels) RIP assays of U2AF65 and Prp19 in the same cells. Anti-U2AF65 or anti-Prp19 IP, vs IgG control IP were used to calculate the mean fold binding enrichment in the indicated RNA regions ±SD. Primers listed in Supplementary Table 2. Primer location in Supplementary Fig.7b.e(Upper panel) shIWS1 rescue by U2AF65α and U2AF65β. Spliced/unspliced RNA ratios ofCDCA5and GUSB, measured by qRT-PCR, as in Fig. 5d. (Middle and Lower panels) RIP assays of U2AF65 and Prp19 in the same cells. Data presented as in figure 5d.fCytosolicCDCA5mRNA levels in the indicated shIWS1-transduced cells were rescued by IWS1 and U2AF65α, as determined by q-RT-PCR.GAPDH-normalizedCDCA5mRNA ±SD. Validation of fractionation in Supplementary Fig.7e.gLysates of NCI-H522 cells, transduced with the indicated constructs, were probed with antibodies, as shown. DM-A and DM-E are the S79/S209AA and S79/S209EE Sororin mutants, respectively.h(Upper panels) Lysates ofKRASandEGFRmutant cell lines, transduced with the indicated constructs, were probed with antibodies as shown. RT-PCR, usingU2AF2exon 1 and 3 primers. (Lower Left panel) Bars show the qRT-PCR-determinedU2AF2E2/E3 ratios in NCI-H522 and NCI-H1299 cells, and in theKRASandEGFRmutant cell lines, relative to the shControl±SD. (Lower Right panel) Bars show the shIWS1-induced percent reduction of ERK-phosphorylation in the same cell lines, normalized to tubulin ± SD.EGFRmutant and non-mutant cells were compared, using a one-way ANOVA. All assays were in triplicate, on three biological replicates. n.s non-significant, *p< 0.05, **p< 0.01, ***p< 0.001, ****p< 0.0001 (one-sided unpairedt-test). Statistical analyses were performed using the one-sided unpaired t -test. d Kaplan-Meier Curves of phosphor-IWS1 and U2AF2 E2/E3 ratios in the LUAD cohort in panel a . Statistical analyses were performed using the one-sided log rank test and Cox’s proportional hazards model. e Heat Maps showing the correlation of IWS1 or SRSF1 with components of the IWS1/U2AF2 pathway in the TCGA LUAD database using log 2 normalized counts. f Heatmaps showing the expression of IWS1 pathway components in the tumors of the GSE13213 dataset. g (Left panel) Heat Maps showing expression of IWS1 pathway components in resected brain metastases and primary lung adenocarcinomas. RNA-seq data for metastatic lesions were derived from the GSE141685 dataset and for primary LUADs from TCGA. (Right upper panel) scRNA-Seq data from GSE123903. Force-directed layout/t-SNE of all metastatic tumor cells isolated from patient-derived mouse xenografts (Laughney et al., 2020 71 ), colored by source, (Right lower panel) Force-directed layout (as in the upper panel) of all xenograft tumor cells colored for z -normalized IWS1 and CDCA5 expression. h Kaplan–Meier curves showing the impact of IWS1, U2AF2 E2/E3 and FGFR2 IIIb/IIIc ratios on patient survival in the indicated patients in the TCGA LUAD database. Statistical analyses were performed as in panel d . Full size image Human LUAD frequently harbors KRAS or EGFR mutations and data presented in this report suggested that lung adenocarcinoma cells harboring EGFR mutations may be more sensitive to the loss of IWS1 than KRAS mutant cells (Figs. 5 , 6 , 7 and Supplementary Fig. 10a ). To identify tumors harboring mutations in these genes, we probed the tumor lysates with monoclonal antibodies, which selectively recognize the G12V and G12D mutants of KRAS and the L858R mutant of EGFR [69] (Fig. 8a ). Comparison of the abundance of IWS1 and phosphorylated IWS1 with the U2AF2 E2/E3 ratio, and with the abundance of Sororin, CDK1, phosphor-CDK1, and Cyclin B1, revealed strong correlations in the entire cohort. However, the correlations were more robust in the EGFR than in the KRAS mutant tumors (Fig. 8b ). Consistent with these data, the abundance of phosphor-IWS1 and the U2AF2 E2/E3 ratio, correlates positively with tumor stage (Fig. 8c ) and negatively with survival in patients with EGFR mutant, but not KRAS mutant tumors (Fig. 8d ). The preceding data were confirmed by IHC, using sequential sections of a commercially available tissue microarray (TMA) of 50 LUAD with paired NAT. The TMA samples were probed with antibodies to p-IWS1, Sororin, p-ERK, p-CDK1, and EGFR ΔE746-A750 (Supplementary Fig. 12b , c ). The results confirmed that the pathway is more active in the tumors, than in NAT (Supplementary Fig. 12d ) and that its activity correlates with tumor stage and grade (Supplementary Fig. 12e , f). More important, the abundance of IWS1 phosphorylation correlates with the abundance of Sororin, phosphor-ERK, and phosphor-CDK1, and the correlations are significantly more robust in the EGFR mutant tumors (Supplementary Fig. 12g ). In addition to confirming the western blot data in our set of LUADs, the IHC data also demonstrate that the activity of the pathway can be monitored in human tumors by IHC. The data generated from the analysis of the tumor samples in our LUAD cohort, and the tumor samples in the TMA, were confirmed by data in publicly available databases. Analysis of LUAD data derived from the Tumor Cancer Genome Atlas (TCGA), revealed correlations between IWS1 or SRSF1, and the U2AF2 E2/E3 ratio, as well as other components of the IWS1 phosphorylation pathway (Fig. 8e ). The U2AF2 E2/E3 ratio and the expression of the CDCA5 mRNA were also significantly higher in tumors expressing high levels of IWS1 (Supplementary Fig. 12h ) and IWS1 expression exhibited a positive correlation with tumor stage, in tumors harboring EGFR but not KRAS mutations (Supplementary Fig. 12i ). Analysis of the molecular signature dataset GSE13213, which focuses on tumor relapse [70] , revealed that the expression of IWS1 , CDCA5 , CDK1 , and CCNB1 (encoding Cyclin B1) was higher in a set of relapsing than in another set of non-relapsing LUADs (Fig. 8f , left panel). Sorting tumors harboring EGFR or KRAS mutations into separate groups, revealed that the activity of the pathway was again higher, only in relapsing tumors with EGFR mutations (Fig. 8f , middle and right panels, Supplementary Fig. 12j ). We conclude that the IWS1 phosphorylation pathway may also promote treatment relapse of lung adenocarcinomas, especially those with EGFR mutations. Analysis of the RNA-seq data in the GSE141685 lung adenocarcinoma dataset of primary tumors and brain metastases revealed that the expression of IWS1 and its targets in the IWS1 phosphorylation pathway was higher in the metastatic tumors (Fig. 8g , Supplementary Fig. 12k ). Importantly, the U2AF2 E2/E3 ratio was also higher in the metastatic tumors, while the IIIb/IIIc FGFR2 transcript ratio was reduced (Supplementary Fig. 12l ), in agreement with our earlier observations, showing that IWS1 phosphorylation promotes FGFR2 exon 8 skipping [22] . The role of the IWS1 phosphorylation pathway in metastasis was additionally supported by the results of single-cell RNA-Seq experiments on tumors, in a patient-derived LUAD mouse model [71] . These results revealed that both IWS1 and CDCA5 are highly expressed in subsets of the disseminated tumor cell (DTC) and incipient metastasis sets of tumor cells (Fig. 8g , right panel). Analysis of the RNASeq data in the TCGA-LUAD dataset, which contains information on cancer-associated mutations, confirmed the link between IWS1 expression and metastatic disease, but also showed that IWS1 is upregulated in metastatic tumors with EGFR , but not KRAS mutations (Supplementary Fig. 12m ). As expected from the preceding data, IWS1 expression, U2AF2 exon 2 inclusion, and FGFR2 exon 8 skipping are indicators of poor prognosis in TCGA patients with lung adenocarcinomas, harboring EGFR , but not KRAS mutations (Fig. 8h ). In addition, EGFR mutations in LUADs in the TCGA and the GSE13213/GSE26939 datasets were associated with worse prognosis, when they occurred in patients with high expression of IWS1 (Supplementary Fig. 12n , o). The AKT/IWS1/ U2AF2 /CDCA5/ERK pathway can potentially be activated by multiple mechanisms in human lung adenocarcinomas. To determine the potential role of genetic changes in the activation of the pathway, we examined the whole-exome sequencing information in the TCGA-LUAD dataset for copy-number variations, point mutations, and genomic fusions involving genes in this pathway (Supplementary Data 1 ). This analysis identified several genetic changes of which the most common was an amplification of the AKT3 gene (Supplementary Fig. 13a ). Gain-of-function mutations targeting AKT1 (E17K, D323Y) were also observed (Supplementary Fig. 13b ). The significance of other mutations (L11F and Q10H, immediately upstream of the RS domain of U2AF65) and the significance of X77 = , a splice-site U2AF2 mutation, is not known. The pathway described in this report is activated by AKT, primarily AKT3, upregulates CDCA5, and is associated with poor prognosis. Here we show that both the high expression of AKT3, the signaling molecule at the initial step of the activation of the pathway, and CDCA5, the signaling molecule at the pathway endpoint, are also associated with poor prognosis (Supplementary Fig. 13c ). These data provide additional support to the importance of this pathway in the pathophysiology of human lung adenocarcinomas. Data presented in this report describe a signaling pathway, which starts with the AKT3-dependent phosphorylation of IWS1 and promotes cell proliferation by regulating the alternative RNA splicing of U2AF2 , the RNA splicing of its target CDCA5 , and the expression of the CDCA5 -encoded protein Sororin. Specifically, IWS1 phosphorylation promotes the inclusion of the alternatively spliced exon 2 in the mature U2AF2 mRNA transcript. Exon 2 encodes the RS domain of the U2AF2 protein product U2AF65, which interacts with several proteins involved in the regulation of RNA metabolism, one of which is the ubuiquitin ligase Prp19. The latter is a member of a splicing complex composed of four core and three accessory polypeptides, which is recruited to RNA Pol II via its interaction with the RS domain of U2AF65. Data in this report confirmed that only the protein encoded by the exon 2-containing splice form of U2AF2 (U2AF65α), which is expressed in cells undergoing AKT-dependent IWS1 phosphorylation, interacts with Prp19. In addition, they showed that the Prp19-interacting protein U2AF65α is required for CDCA5 mRNA processing, Sororin expression, cell cycle progression through G2/M, and cell proliferation. Sororin is phosphorylated by ERK, and following phosphorylation, promotes the activation of ERK by indirect and poorly understood mechanisms. We should add that the Sororin-dependent phosphorylation of ERK plays a dominant role in ERK regulation, as inhibition of the IWS1 phosphorylation pathway significantly inhibits the activation of ERK by EGFR mutations and has a major impact in the biology of lung adenocarcinomas harboring such mutations. Importantly, the IWS1 phosphorylation pathway summarized here is an integral component of the cell cycle machinery, as it does not only regulate the cell cycle, but is also cell cycle-regulated. The results of our earlier studies, combined with the data in this report, show that a given RNA splicing regulator may modulate alternative RNA splicing of different target genes by different mechanisms. Our previous findings had shown that the abundance of IWS1 and IWS1 phosphorylation regulates the alternative RNA splicing of FGFR2 by promoting the exclusion of the alternatively spliced exon 8 from the mature transcript. Here we show that IWS1 and IWS1 phosphorylation promote the inclusion of alternative spliced exons in the mature transcripts of several genes. Moreover, although the SETD2-dependent H3K36 trimethylation is required for alternative RNA splicing in both cases, the effector complexes nucleated by H3K36me3 differ. Thus, whereas the H3K36me3 reader responsible for exon exclusion from the FGFR2 mRNA is MRG15, the H3K36me3 reader for exon inclusion in the U2AF2 mRNA is the p52 isoform of LEDGF. Also, whereas H3K36/MRG15 recruits the spliceosomal factor PTB for the alternative splicing of FGFR2 , H3K36/LEDGF (p52) recruits SRRSF1 for the alternative splicing of U2AF2 . Currently, we do not know why the two types of genes respond differently to the IWS1 phosphorylation-induced histone H3K36 trimethylation. One possibility is that cis-acting elements in the RNA facilitate the binding of factors, which could synergize with specific H3K36me3 readers and associated proteins. This is supported by findings reported here, which show that RNAs undergoing IWS1-dependent exon inclusion, including the U2AF2 mRNA, contain sites that may be recognized by SRSF1. Alternatively, there may be differences in the epigenetic marks responsible for the selection of H3K36me3 readers and reader-associated factors in different genes. We should add here that our earlier studies and data in this report show that not only both mechanisms have a role in human cancer, but they may also be active simultaneously in the same cancer. Another important observation presented in this report is that mRNA splicing is a process that is regulated at multiple levels. Thus, the alternative splicing of U2AF2 is regulated directly by the IWS1 phosphorylation-dependent abundance of histone H3K36me3 marks in the body of the U2AF2 gene. However, by regulating the alternative splicing of a basic RNA splicing factor, this process introduces a new layer of RNA splicing regulation, which depends in part on the differential binding of U2AF65 to yet another splicing factor, Prp19. The binding between these factors is required for the efficient splicing of CDCA5 and perhaps other genes. The reason for the multilayered control of RNA splicing by a single RNA splicing regulator could be that this allows a limited number of available pathways to converge in different combinations for the differential modulation of a large number of RNA splicing events. This may be critical for the fine-tuning of the global regulation of RNA splicing under different physiological conditions. We should add here that although the effects of the RS domain-deficient U2AF65 on RNA splicing may be global, they are selective, affecting the RNA splicing of some, but not all the genes. One of the factors that determine the specificity in the pathway described here could be the binding of Prp19, but this question remains to be addressed. The IWS1 phosphorylation pathway described in this report plays a critical role in cell cycle progression by regulating the RNA splicing of CDCA5 and the abundance of the CDCA5 -encoded protein Sororin. The latter is one of the seven members of the cohesin complex, a ring-like structure, which holds the sister chromatids together during metaphase [72] . Defects in this complex activate the spindle assembly checkpoint, arresting progression through G2/M [73] . This explains the partial G2/M arrest induced by the CDCA5 mRNA processing block associated with the downregulation of IWS1 expression and/or phosphorylation and with the RS domain-deficient U2AF65β. However, the downregulation of CDCA5/Sororin may interfere with additional G2/M-associated processes, such as transcription of genes contributing to progression through the G2/M phase of the cell cycle. Data presented in this report show that Sororin expression and/or phosphorylation, promotes the expression of CCNB1 and CDK1 at both the RNA and protein levels. In addition, the abundance of the CDCA5 mRNA exhibits very strong correlations with the abundance of the CCNB1 and CDK1 mRNAs, in the TCGA datasets of human lung adenocarcinomas. These observations indicate that the induction of cyclin B1 and CDK1 by Sororin is regulated at the RNA level, most likely at the level of transcription. A potential mechanism for the transcriptional regulation of CCNB1 and CDK1 by Sororin was suggested by earlier studies showing that the Cohesin complex interacts with the Mediator complex and that Mediator–Cohesin complexes are loaded by the NIBPL Cohesin loading factor to enhancers and core promoters of target genes. Enhancer and core promoter-associated complexes promote loop formation between these segments and regulate transcription [74] . The contribution of this and other mechanisms on the regulation of CCNB1 and CDK1 expression is under investigation. The information discussed in the preceding paragraph describes a dominant mechanism by which the IWS1 phosphorylation pathway regulates cell cycle progression and cell proliferation. Given that the cell cycle is an integrated system and that cell cycle regulatory mechanisms tend to also be cell cycle-regulated, we examined whether the expression and phosphorylation of IWS1, the RNA splicing of U2AF2 , and the expression of Sororin fluctuate as the cells progress through the cell cycle. The results revealed that the abundance of these molecules and the RNA splicing of U2AF2 indeed fluctuate in a cell cycle-dependent fashion, and confirmed that the regulation of RNA splicing by IWS1 is an integral component of the cell cycle machinery. The fluctuation of the activity of the IWS1 phosphorylation pathway during cell cycle progression is due to the fluctuating levels of IWS1 mRNA, protein, and protein phosphorylation. The latter may be due to cell cycle-dependent changes in the activity of AKT. Earlier reports had indeed shown that CDK2 is activated in S phase by interacting with cyclin A2, and that following activation, phosphorylates AKT at Ser477/Thr479, enhancing its activity [75] . To the changing levels of IWS1 expression and phosphorylation, we should add that the abundance of some core splicing factors also fluctuates with the cell cycle. Our working hypothesis therefore is that the activity of the IWS1 phosphorylation pathway may fluctuate during the cell cycle, due to a combination of cell cycle-dependent processes. An important component of the cell cycle regulatory mechanisms initiated by the AKT-dependent phosphorylation of IWS1 is a positive feedback loop between ERK and Sororin. ERK phosphorylates Sororin and the phosphorylated Sororin promotes the phosphorylation of ERK. How the ERK-phosphorylated Sororin promotes the phosphorylation and activation of ERK is currently unknown. Our working hypothesis is that the phosphorylation and activation of ERK are due to signals induced by the interaction of Sororin with its partners in the cohesin complex. If this is the case, the cell may use this mechanism to sense the successful progression from prometaphase to metaphase, in order to activate a molecular switch, which enhances the phosphorylation of Sororin, facilitating entry into, and progression through the G2/M phase of the cell cycle. One of the most important findings presented in this report is the link between the AKT3/IWS1/U2AF2/CDCA5/ERK pathway and the biology of lung adenocarcinomas harboring EGFR mutations. The first surprising observation was the significant downregulation of the phosphorylation of ERK, induced by the knockdown of IWS1 in lung adenocarcinoma cell lines with EGFR mutations, and to a lesser extent KRAS mutations. Subsequent observations confirmed that the knockdown of IWS1 had a major impact on the proliferation of lung adenocarcinoma cell lines, particularly those with EGFR mutations. Moreover, studies on 40 lung adenocarcinomas from the OSU tumor bank and 50 lung adenocarcinomas in commercially available tissue microarrays showed that the IWS1 phosphorylation pathway is active in primary human tumors. More important, these data also revealed that the activity of the pathway correlates positively with tumor grade and stage, and negatively with patient survival, selectively in tumors harboring EGFR mutations. These observations were also in agreement with data generated from the meta-analysis of lung adenocarcinoma datasets. Meta-analysis of these datasets showed that the activity of the IWS1 phosphorylation pathway selectively correlates not only with tumor grade, tumor stage, and patient survival, but also with metastasis and with tumor relapse following treatment. Collectively, these data suggest that the AKT3/IWS1/U2AF2/CDCA5/ERK pathway is associated with less differentiated, more invasive, and more metastatic tumors, and perhaps with resistance to EGFR inhibitors. Based on these findings, we propose two translational applications for the IWS1 phosphorylation pathway described in this report: (a) the expression and phosphorylation of IWS1, the alternative splicing of U2AF2 , and the gene expression program initiated by these processes, can be used as biomarkers to stratify patients for treatment. (b) Treatment with inhibitors of the EGFR pathway, in combination with AKT1/AKT3 inhibitors or decoy RNA oligonucleotides targeting U2AF2 RNA splicing, may enhance the therapeutic potential of EGFR pathway inhibition and may prevent the emergence of treatment-resistant clones. In conclusion, the data in this report describe an important pathway that links cell cycle-regulated AKT activity to RNA splicing and cell cycle regulation. More important, this process is active in a significant fraction of human lung adenocarcinomas, and its activity is associated with poor prognosis selectively in patients with lung adenocarcinomas harboring EGFR mutations. The activity of this pathway therefore, provides a precision medicine biomarker, which may be used to stratify human lung adenocarcinomas and inform the optimal treatment strategy. Cells, culture conditions, growth factors, and inhibitors NCI-H522, NCI-H1299, and HEK-293T cells were grown in Dulbecco’s modified Eagle’s medium (DMEM) (Sigma-Millipore, Cat No. D5796) supplemented with penicillin/streptomycin (Corning, Cat No. 30-002-CI), nonessential amino acids (Corning, Cat No. 25-025-CI), glutamine (Corning, Cat No. 25-005-CI), plasmocin 2.5 ng/μL (Invivogen, Cat No. ant-mpp), and 10% fetal bovine serum. A549, NCI-H460, NCI-H1975, PC-9, NCI-H1650 and HBEC hTERT cells were grown in similarly supplemented Roswell Park Memorial Institute 1640 (RPMI 1640) medium (Sigma-Millipore, Cat No D8758). Cell lines were periodically checked for mycoplasma, using the PCR mycoplasma detection kit (ABM, Cat No. G238) and they were used for up to five passages. All experiments were carried out in mycoplasma-free cultures. IGF1 (Cell Signaling, Cat. 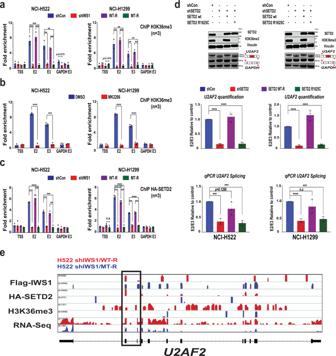No. 8917) (20 ng/mL), was used to stimulate NCI-H522 or NCI-H1299 cells that had been serum-starved for 24 h. Cells were treated with IGF1 for up to 4 h. To inhibit AKT in cells growing in complete media, we treated them with the AKT inhibitor MK2206 (MERCK) (5 μM) for 4 h. At this concentration, MK2206 inhibits all three AKT isoforms. siRNAs, shRNAs, expression constructs, and site-directed mutagenesis siRNAs, shRNAs, and expression constructs are described in Supplementary Table 3 . Fig. 3:U2AF2Exon 2 inclusion, induced by IWS1 phosphorylation at Ser720/Thr721, depends on H3K36 trimethylation by SETD2. aChIP assays showing the abundance of H3K36me3 in the indicated NCI-H522 (left) and NCI-H1299 (right) cells. Bars show the mean fold enrichment in H3K36me3 (anti-H3K36me3 IP, vs IgG control IP) in the indicated regions of theU2AF2gene, in shControl, shIWS1, shIWS1/WT-R and shIWS1/MT-R cells ±SD. Data were normalized relative to the input (2%).bChIP assays showing the abundance of H3K36me3 in the indicated NCI-H522 (left) and NCI-H1299 (right) cells, treated with MK2206 (5μM) or DMSO. The bars show the mean fold enrichment of H3K36me3 (anti-H3K36me3 IP, vs IgG control IP) in the indicated regions of theU2AF2gene, ±SD. Data were normalized relative to the input (2%).cChIP assays showing the binding of HA-SETD2 in the indicated NCI-H522 (left) and NCI-H1299 (right) cells, transduced with a lentiviral HA-SETD2 construct. The bars show the mean fold enrichment in SETD2 binding (anti-HA IP, vs IgG control IP) ±SD. Data were normalized relative to the input (2%). The expression of HA-SETD2 is shown in Supplementary figure 4a.d(Upper panel) Lysates of NCI-H522 (left) and NCI-H1299 (right) cells transduced with the indicated constructs, were probed with the antibodies, as shown. RT-PCR addressingU2AF2exon 2 splicing in the same cells. (Middle panel)GAPDH-normalized E2 and E3 bands in the RT-PCR experiment above, were used to calculate the E2/E3 ratio±SD. (Lower panel) Ratio of theU2AF2exons 2 and 3 levels in the same cells ±SD, as determined by quantitative RT-PCR. E2/E3 ratio is shown relative to shControl (value = 1). All experiments had three biological replicates, all done in triplicate. n.s non-significant, *p< 0.05, **p< 0.01, ***p< 0.001, ****p< 0.0001 (one-sided unpairedt-test).eSnapshots of the integrative genomic viewer showing the ChIP-Seq-determined distribution of Flag-IWS1, HA-SETD2, and histone H3K36me3, inU2AF2. Parallel snapshots show the distribution of RNA reads in the RNA-seq experiment. Scale represents reads per million (RPM). Snapshots of peaks detected in the two biological replicates are shown. Black box highlightsU2AF2exons 2, 3 and adjacent regions. cDNA copies of the U2AF2 splice variants α and β were amplified by RT-PCR, from NCI-H522 shControl and NCI-H522 shIWS1 cells, respectively. The amplified cDNAs were electrophoresed in 1% agarose gels and they were gel-purified using the NucleoSpin Gel and PCR Clean-Up kit (M&N, Cat. No. 740609.50). The purified cDNAs were cloned in the pENTR/D-TOPO cloning vector (Invitrogen, Cat. No. 45-0218). Subsequently, they were transferred by recombination from the pENTR/D-TOPO clones to pLx304-V5-DEST (Addgene #25890), using standard Clonase II LR mix (Thermofisher, Cat No 11791100). The Gateway LR reaction was incubated at room temperature overnight. pDONR201-p52/LEDGF was purchased from the DNAsu Plasmid Repository (DNAsu Plasmid Repository Clone: HsCD00000034). p75/LEDGF cDNA was amplified by RT-PCR from NCI-H522 shControl cells and was cloned into pENTR/D-TOPO cloning vector. Cloning to the pENTR/D-TOPO Vector and transfer to the PLX-304-V5-DEST vector were carried out as described above for the U2AF2 cDNA clones. Site-directed mutagenesis was carried out using standard PCR-based techniques. Briefly, pairs of overlapping oligonucleotide primers, harboring the desired mutation, were used to amplify plasmids containing the genes we wished to mutagenize. To remove the original plasmid from the amplified reaction mix, we incubated it with 2 μL of the 6-methyladenine-dendent restriction endonuclease DpnI,(NEB, Cat. No R0176) at 37 °C for 4 h. Subsequently, the DNA in the reaction mix was purified, using the NucleoSpin Gel and PCR Clean-Up kit. At the end, DH5-alpha Electrocompetent Escherichia coli (NEB, Cat. No. C2986) were transformed with 5 μL of the purified product, using an Eppendorf Eporator® (Eppendorf, Cat. No. 4309000027). All the mutagenized constructs were sequenced in the Genomic Shared Resource (GSR) of The Ohio State University ( https://cancer.osu.edu/for-cancer-researchers/resources-for-cancer-researchers/shared-resources/genomics ), prior to use. The primers we used for all the mutagenesis experiments in this report are listed in Supplementary Table 2 . Transfections and infections Retroviral constructs were packaged by transient transfection in 293T cells, in combination with ecotropic (Eco-pac) or amphotropic (Ampho-pac) packaging constructs. Lentivirus constructs were also packaged in HEK-293T cells by transient transfection in combination with the packaging constructs psPax2 (Addgene #12260) and pMΔ2.G (Addgene #12259). Transfections were carried out using 2× HEPES Buffered Saline (Sigma, Cat. No 51558) and CaCl 2 precipitation. Forty-eight hours later, virus-containing culture media were collected and filtered. Infections were carried out in the presence of 8 μg/mL polybrene (Sigma, Cat. No. 107689). Depending on the selection marker in the vector, 48 h from the start of the exposure to the virus, cells were selected for resistance to puromycin (Gibco, Cat. No. A11138) (10 μg/mL), G-418 (Cellgro, Cat. No. 30-234) (500 μg/mL), or blasticidin (Gibco, Cat. No A1113903) (5 μg/mL). Cells infected with multiple constructs, were selected for infection with the first construct, prior to the next infection. Transfection of lung adenocarcinoma cell lines with siRNAs (20 nM final concentration) was carried out, using the Lipofectamine 3000 Transfection Reagent (Invitrogen, Cat. No. 13778) and Opti-MEM Reduced Serum Medium (Gibco, Cat. no. 11058021), according to the manufacturer’s protocol. Cell proliferation assay, cell cycle analysis, and FACS-sorting of cells in different phases of the cell cycle shControl, shIWS1, shIWS1/CDCA5 WT rescue, shIWS1/CDCA5 S79A/S209A mutant rescue, and shIWS1 CDCA5 S79E/S209E mutant rescue cells were plated in triplicate in 12-well tissue culture plates. Given that the growth rates of these cell lines differ, they were plated at different densities (NCI-H522 8000 cells/well, NCI-H1299 5000 cells/well, H1975 5000 cells/well, and A549 8000 cells/well). Cell proliferation of cells growing under normal culture conditions was monitored every 6 h, using the Incucyte S3 Live-Cell Imaging and Analysis System (Essen Biosciences, Ann Arbor, MI). All cell lines were monitored for 7 days, with the exemption of the NCI-H1975 cell line, which was monitored for 12 days. Images were captured and analyzed using the Incucyte confluence masking software (Essen Biosciences, Ann Arbor, MI), which calculates the surface area occupied by the growing cells, as a percentage of the total surface area of the well at sequential time points. Confluence monitoring was optimized for each cell line to minimize background. To ensure an unbiased analysis, the optimization parameters determined for a given cell line were also applied to all the derivatives of that cell line. To determine the cell cycle distribution of exponentially growing cells, semiconfluent cultures were harvested by trypsinization and the cell pellet was resuspended in 700 μL of PBS and fixed by adding 2.8 mL of ice-cold ethanol. The ethanol-suspended cells were kept at −20 °C overnight. Following two washes with 1× PBS, the fixed cells were stained with propidium iodide (Propidium Iodide (1:2500)) (Invitrogen, Cat. No. P3566), 0.1 mg/mL RNAse A (Invitrogen, Cat. No. 12091-039), and 0.05% Triton X and incubated in the dark at 37 °C for 30 min. 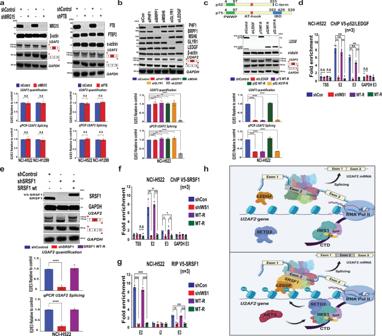Subsequently, the cells were analyzed on a BD FACS Calibur v2.3 Flowcytometer (BD Biosciences, San Jose, CA). All the experiments were performed in triplicate and they were analyzed, using the FlowJo v9.3.3 software. The raw data obtained from this analysis can be found in Supplementary Table 4 . Fig. 4: The regulation of the alternative splicing of theU2AF2exon 2 by IWS1 and IWS1 phosphorylation, depends on the p52 isoform of the H3K36me3 reader LEDGF and its splicing partner SRSF1. a(Upper panel) Lysates of the indicated cells were probed with antibodies, as shown. RT-PCR addressing exon 2U2AF2splicing in the same cells. (Middle and Lower Panels)U2AF2 E2/E3±SD, was determined by quantification of the RT-PCR results and by qRT-PCR.b(Upper Panel) Lysates of NCI-H522 cells transfected with the indicated siRNAs, probed with antibodies, as shown. RT-PCR addressing exon 2U2AF2splicing. (Middle and Lower Panels)U2AF2 E2/E3±SD, was determined by quantification of the RT-PCR results and by qRT-PCR.c(Upper panel) Domains of the p52 and p75 LEDGF isoforms (see Ferris et al., 201050). (Middle panel) Western blot of the indicated NCI-H522 cells, probed for LEDGF expression and RT-PCR, addressingU2AF2exon 2 splicing in the same cells. (Lower panels)U2AF2 E2/E3ratio ±SD, was determined by quantification of the RT-PCR results and by qRT-PCR.dChIP of p52/LEDGF in NCI-H522 cells, transduced with V5-p52/LEDGF. Mean fold enrichment in p52/LEDGF binding (anti-V5 IP, vs IgG control IP) to the indicatedU2AF2regions±SD. V5-p52/LEDGF expression, in figure S5G.e(Upper panel) Immunoblotting, showing SRSF1 expression in the indicated NCI-H522 cells. RT-PCR addressingU2AF2exon 2 splicing. (Lower panels)U2AF2 E2/E3ratio ±SD, was determined by quantification of the RT-PCR results and by qRT-PCR.fSRSF1 ChIP in the indicated V5-SRSF1-transduced NCI-H522 cells. Mean fold enrichment in SRSF1 binding (anti-V5 IP, vs IgG control IP) to the indicatedU2AF2regions±SD. V5-SRSF1 expression in Supplementary figure S6b.gRIP, addressing SRSF1 binding toU2AF2RNA in panelfcells. Mean fold enrichment in SRSF1 binding (anti-V5 IP, vs IgG control IP) in the indicatedU2AF2regions ±SD. All assays were done, using three biological replicates, in triplicate. n.s non-significant, *p< 0.05, **p< 0.01, ***p< 0.001, ****p< 0.0001 (one-sided unpairedt-test).hPhosphorylation of IWS1 recruits SETD2 in CTD of RNA Pol II. SetD2 trimethylates histone H3K36 co-transcriptionally. p52/LEDGF and its partner SRSF1, bind histone H3K36me3 promoting exon 2 inclusion in the matureU2AF2transcript. The analysis was performed in the Flow Cytometry Shared Resource of the Ohio State University ( https://cancer.osu.edu/for-cancer-researchers/resources-for-cancer-researchers/shared-resources/flow-cytometry ). To separate cells in different phases of the cell cycle for further analysis, 2 × 10 6 exponentially growing NCI-H1299 cells were harvested by trypsinization, counted, and resuspended in DMEM, to a final concentration of 5 × 10 5 cells/mL. Following this, cells were stained by adding 2 μL/mL Vybrant™ DyeCycle™ Ruby Stain (Thermo Fisher, Cat. No. V10309) and by incubating them in the dark at 37 °C for 30 min. The stained cells were sorted based on their DNA content, using a BD FACS Aria III cell sorter (BD Biosciences, San Jose, CA). Cellular fractions enriched for cells in G1, S, and G2/M were harvested for protein, RNA, and chromatin analyses. For protein extraction, cells were lysed in RIPA lysis buffer (LB) and processed for immunoblotting. For RNA extraction, we used the PureLink RNA Kit. Extracted RNA was used for RT-PCR and qRT-PCR analyses, as described in this report. Chromatin analyses were performed using ChIC. The antibodies and primer sets used are described in Supplementary Tables 1 and 2 , respectively. Cell transformation assay Cell transformation assays in immortalized HBEC hTERT were performed using the Cell Transformation Assay Kit-Colorimetric (Abcam Cat No. ab235698). Based on the manufacturer’s protocol, two layers of agarose were made (base and top layer). Prior to the initiation of the experiment, we performed a cell-dose curve by using seven serial dilutions of cells (twofold) and incubating them for 4 h at 37 °C with WST working solution. After that, the absorbance at 450 nm was determined and the cell-dose curve was calculated \(y=\alpha x+\beta\) , using linear regression on GraphPad Prism 8.4. In order to perform the assay, after solidification of the base agarose layer, 2.5 × 10 4 HBEC hTERT cells per condition were mixed with top agarose layer in 10× DMEM solution and plated in a 96-well plate, in triplicates along with blank wells. The cells were then plated for 7 days at 37 °C and monitored for colony formation. After 7 days, the cells were imaged in the Incucyte live-cell imager using the 20× lens. Then, the cells were incubated for 4 h on WST working solution at 37 °C. The absorbance at 450 nm was determined with a plate reader. Regarding the analysis, the average of the blank wells was subtracted from all the readings of the experimental conditions. Then, the final number of the transformed cells was calculated by inserting the corrected values in the cell-dose curve created prior to the experiment. Library preparation and RNA-seq Total RNA was isolated from shControl, shIWS1, shIWS1/WT-R, and shIWS1/MT-R NCI-H522 cells, using the PureLink RNA Kit (Invitrogen Cat No 12183018A). RNA samples were analyzed on Advanced Analytical Fragment Analyzer, using an RNA kit for integrity check and quantification. About 100–500 ng of total RNA from each sample was used as input for library preparation with the Illumina TruSeq stranded mRNA Library Preparation Kit (Cat. No. RS-122-2101) and they were individually indexed. Libraries were quantified on Fragment Analyzer using a next-generation sequencing (NGS) kit and the libraries of all the samples were pooled in equal molar concentration. The pooled library was sequenced on an Illumina HiSeq 2500 platform with Rapid V2 chemistry and 100-bp paired-end reads. Sequencing results were demultiplexed with bcl2fastq and compressed. Demultiplexed fastq file pairs from each sample were used for analysis. The whole procedure was performed in the Tufts University Core Genomic Facility (TUCF- http://tucf-genomics.tufts.edu ). All RNA-Seq experiments were performed in duplicate, and average depth of sequenced samples was 37.5M (±5M fragments). Data preprocessing and alignment was conducted as previously described [76] . RNA-Seq libraries were quality-checked using FastQC ( www.bioinformatics.babraham.ac.uk/projects/fastqc/ ). Adapters and sequence contaminants were detected and removed using an in-house-developed algorithm and additional software such as the Kraken suite and Cutadapt [77] . Paired-end reads were aligned against the human reference genome (GRCh38/hg38) with GSNAP [78] spliced aligners. For gene and transcript annotation, we utilized Ensembl v85 reference database [79] . Differential gene expression and alternative RNA splicing Gene expression and exon-level expression was calculated by counting reads overlapping meta-gene and exon features using featureCounts [80] . DESeq [81] and DEXSeq [38] were employed to address differential gene expression and differential exon usage, respectively. Differential gene expression analysis We performed differential gene expression analyses using R package DESeq, which utilizes a generalized linear model (GLM) and is applied directly to raw read counts. When we compared the transcriptomes of shIWS1 and shControl cells, we identified 1357 differentially expressed genes ( p value ≤ 0.01, FDR ≤ 0.2), and when we compared the transcriptomes of shIWS1/WT-R and shIWS1/MT-R cells, we identified 417 differentially expressed genes ( p value ≤ 0.01, FDR ≤ 0.2). Differential exon usage DEXSeq employs a GLM to model the differential exon usage between sample groups. Pairwise comparison of the transcriptomes of shIWS1 and shControl cells with DEXSeq identified 1,434 differentially employed exons, assigned to 851 genes (FDR ≤ 0.05). Pairwise comparison of the transcriptomes of shIWS1/WT-R and shIWS1/MT-R cells, identified 436 differentially utilized exons, assigned to 273 genes (FDR ≤ 0.05). Detailed lists of differentially expressed genes and differentially used exons, are provided in supplementary files. In both DESeq and DEXSeq analyses, false discovery rate (FDR) was controlled with the Benjamini–Hochberg procedure [82] . One hundred and sixty-five genes were identified as both differentially expressed and alternatively spliced when we compared the transcriptomes of shIWS1 and shControl cells. Similarly, transcriptomic comparison of shIWS1/WT-R and shIWS1/MT-R cells identified 44 differentially expressed and alternatively spliced genes. Gene-set enrichment analysis (GSEA) For this analysis, we used the GSEA v2.0.13 software. All the gene set files were downloaded from GSEA website ( www.broadinstitute.org/gsea/ ). Enrichment maps were used for visualization of the GSEA results. Enrichment score and FDR values were applied to sort pathways enriched after gene set permutations were performed 1000 times for the analysis. Functional analysis of alternative RNA splicing events Log 2 fold-change values of alternative spliced genes whose RNA splicing is differentially affected in shIWS1 vs shControl and shIWS1/WT-R vs shIWS1/MT-R NCI-H522 cells, were imported in the RStudio framework (V 3.5.2) for the GO analysis. GO analysis was performed, using the Bioconductor GOfuncR software [83] . Alternatively spliced genes were annotated, according to their biological process. For each biological process, the number of associated genes and combined score, which is the absolute value of the sum of the Log 2 fold change values of each gene associated with the biological process, were also calculated. Subcellular fractionation About 5 × 10 6 cells were trypsinized, following two washes with ice-cold PBS. Harvested cells were centrifuged at 1200 × g for 5 min and the pellet was resuspended in 1 mL of PBS and aliquoted into two equal fractions, one for protein and the other one for RNA isolation. In the first fraction, the cells were lysed using a Triton X-100 cytosolic LB1 {(50 mM Tris-HCL (pH 7.5), 20 mM NaCl, 1 mM EDTA, 0.5% NP-40, 0.25% Triton X-100, 10% Glycerol, and 1 mM DTT) and fresh 1× Halt™ Protease and Phosphatase Inhibitor Cocktails (Thermofisher, Cat. No 78444)}. Lysates were rotated for 10 min at 4 °C, and following this, they were clarified by centrifugation at 14,000 × g for 6 min. The supernatant, containing the cytosolic protein fraction, was collected for downstream applications. The precipitated nuclear fraction was further treated with LB2 {(10 mM Tris-HCL (pH 7.5), 20 mM NaCl, 1 mM EDTA, 0.5 mM EGTA, and 1 mM DTT) and fresh 1× Halt™ Protease and Phosphatase Inhibitor Cocktails}. The LB2 lysates were again clarified by centrifugation at 12,000 × g for 6 min. The pellet containing the nuclei, was further lysed with LB3 {(10 mM Tris-HCL (pH 7.5), 100 mM NaCl, 1 mM EDTA, 0.5 mM EGTA, 0.1% (w/v) sodium deoxycholate, and 0.5% (v/v) N-lauroylsarcosine) and fresh 1× Halt™ Protease and Phosphatase Inhibitor Cocktails}. The LB3 lysates were sonicated and clarified by centrifugation at 21,000 × g for 15 min. To validate the fractionation, nuclear and cytosolic fractions were analyzed by immunoblotting for the abundance of Lamin A/C and GAPDH. The cells in the second fraction, were washed twice with TD buffer (135 mM NaCl, 5 mM KCl, 0.7 mM Na 2 HPO 4 , and 25 mM Tris-HCl) and then lysed using TD/1% NP-40/RVC (Ribonucleoside-Vanadyl Complex, NEB, Cat. No. S1402) in the presence of the Recombinant Ribonuclease Inhibitor RNaseOUT™ (Thermo Fisher, Cat. No. 10777019). Following incubation on ice for 10 min, and centrifugation at 21,000 × g for 1 min, the supernatant (cytosolic fraction), was aspirated and kept on ice. The nuclear fraction was washed twice with TD/0.5% NP-40/RVC. The RNA from both fractions was isolated using Trizol and a mixture of phenol–chloroform–isoamyl alcohol and it was precipitated with ethanol at −80 °C overnight. cDNA was synthesized from 1.0 μg of total RNA, using oligo-dT priming and the QuantiTect Reverse Transcription Kit. Quantitative RT-PCR was carried out as described in the following section. Immunoprecipitation [84] , immunoblotting, and image acquisition and utilization For the immunoprecipitation experiments in this report, we first fractionated cell lysates into nuclear and cytoplasmic fractions, using the protocol described under cell fractionation. LB3 nuclear lysates were sonicated and clarified by centrifugation at 21,000 × g for 15 min. About 300 μL of the clarified lysates were added to Magnetic beads-Antibody conjugates, which were prepared as follows. Pierce™ Protein A/G Magnetic Beads (Thermofisher, Cat. No 88803) were washed 3 times, 5 min each, with LB3. Following overnight incubation at 4 °C with the immunoprecipitating antibody or the Mouse Isotype Control antibody (Thermofisher, Cat. 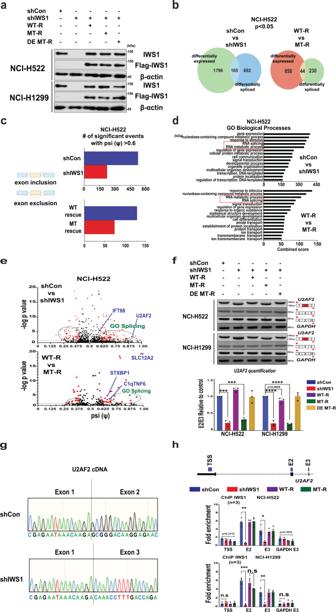No 10400 C), the bead–antibody conjugates were again washed multiple times with LB3. Following the addition of 300 μL of the clarified lysates to the antibody–bead conjugates, the mixture was incubated at 4 °C overnight. The agarose bead-bound immunoprecipitates were washed five times, 5 min each, with LB3, and they were electrophoresed (20 μg protein per lane) in SDS-PAGE. Following electrophoresis, proteins were transferred to polyvinylidene difluoride (PVDF) membranes in 25 mM Tris, 192 mM glycine. Immunoprecipitated proteins were detected by probing the membranes with the relevant antibodies, as described in the following paragraphs. To reduce the IgG heavy- and light-chain signal, V5-tagged and endogenous U2AF65 were immunoprecipitated using a mouse monoclonal antibody and they were detected with a rabbit monoclonal U2AF65 antibody. Fig. 1: IWS1 expression and/or phosphorylation regulate alternative mRNA splicing. aWestern blots of NCI-H522 and NCI-H1299 cell lysates, transduced and probed with the indicated constructs and antibodies.bOverlaps between differentially-expressed and differentially spliced genes in the indicated groups (q< 0.05).cBar graphs of alternative splicing events with exon inclusion. The comparisons were limited to alternative splicing events with a percentage of the alternatively spliced exon spliced in (psi/ψ) >0.6 and apvalue < 0.05.dGO analysis of statistically significant alternative splicing events in the indicated groups (p< 0.05). Red boxes highlight gene sets involved in the regulation of RNA processing.eVolcano plots of all the exon inclusion and exclusion alternative splicing events, detected by DEXseq in the indicated groups. The statistically significant events (p< 0.05) with a percentage spliced in (psi/ψ) level of >0.6 or <0.4 are shown in red. Statistically significant events in the GO functions RNA splicing or RNA metabolic processes are shown in green. Alternatively spliced IWS1 targets validated in this report are shown in blue.f(Upper panel) RT-PCR ofU2AF2in the indicated NCI-H522 and NCI-H1299 cells, using primers mapping in exons 1 and 3, 3 and 5, and 8 and 10 (control).GAPDHwas used as the loading control. TheU2AF2 E2/E3ratio was calculated from the GAPDH-normalized levels of the RT-PCR products. The bars show the mean ratio ± SD in the indicated NCI-H522 and NCI-H1299 cells relative to shControl.gSequencing chromatograms of the two alternatively splicedU2AF2RNA transcripts.h(Upper) UCSC browser snapshot showing exons 1, 2, and 3 of the humanU2AF2gene. The map position of the PCR primer sets used in the ChIP experiments in this figure is indicated by blue marks. (Lower) ChIP assays of IWS1 on theU2AF2andGAPDHgenes in shControl, shIWS1 shIWS1/WT-R and shIWS1/MT-R NCI-H522 and NCI-H1299 cells. Bars show the mean fold enrichment (anti-IWS1 IP, vs IgG control IP) in IWS1 binding, in shIWS1 relative to shControl cells or in shIWS1/MT-R relative to shIWS1/WT-R cells ±SD. Data were normalized relative to the input (2%). All assays were done in triplicate, on three biological replicates. n.s: non-significant, *p< 0.05, **p< 0.01, ***p< 0.001, ****p< 0.0001 (one-sided unpairedt-test). Antibodies used for immunoprecipitation are listed in Supplementary Table 1 . The detailed protocol can be found in the online protocol repository [84] . For immunoblotting, cells were lysed using a RIPA LB {50 mM Tris (pH 7.5), 0.1% SDS, 150 mM NaCl, 5 mM EDTA, 0.5% sodium deoxycholate, 1% NP-40, and fresh 1× Halt™ Protease and Phosphatase Inhibitor Cocktails (Thermofisher, Cat. No 78444)}. Lysates were sonicated twice for 30 s and clarified by centrifugation at 18,000 × g for 15 min at 4 °C. The clarified lysates were electrophoresed (20 μg protein per lane) in SDS-PAGE. Electrophoresed lysates were transferred to PVDF membranes (EMD Millipore Cat No. IPVH00010) in 25 mM Tris and 192 mM glycine. Following blocking with 5% nonfat dry milk in TBS and 0.1% Tween-20, the membranes were probed with antibodies (at the recommended dilution), followed by horseradish peroxidase-labeled secondary antibodies (1:2500), and they were developed with Pierce ECL Western Blotting Substrate (Thermo Scientific, cat. no 32106). The antibodies used for western blotting are listed in Supplementary Table 1 . Western blot images were captured, using the Li-Cor Fc Odyssey Imaging System (LI-COR Biosciences, Lincoln, NE). For protein ladder detection, we used the 700-nm channel and for protein band detection, we used the chemiluminescence channel. Data were collected using a linear acquisition method. All images in this report were captured with the same protocol in order to ensure the comparability of the results from different experiments. Images were exported in high-quality image files (600-dpi png files) and they were processed with the X Illustrator 2020 (Adobe, San Jose, CA) for figure preparation. The summary figures in Figs. 4 h, 6j, and Supplementary Fig. 9c were designed in Bio Render using a student plan promo (legacy), and include content from Biorender ( https://biorender.com/terms/ ). qRT-PCR and RT-PCR Total cell RNA was extracted using the PureLink RNA Kit (Invitrogen, Cat. No 12183018A). cDNA was synthesized from 1.0 μg of total RNA, using oligo-dT priming and the QuantiTect Reverse Transcription Kit (QIAGEN, Cat No. 205310). Gene and exon expression was measured by quantitative RT-PCR, using the iTaq™ Universal SYBR® Green Super mix (Biorad, Cat No. 1725121) and a StepOne Plus qRT-PCR instrument (Thermofisher). qRT-PCR experiments were performed with three biological replicates in triplicate. Data were normalized to internal controls hGAPDH mRNA, or human 18S rRNA . The primer sets used for all the real-time PCR assays are listed in Supplementary Table 2 . Chromatin immunoprecipitation (ChIP) Attached cells were washed with PBS and then treated with 1% formaldehyde (Sigma, Cat. No F8775) for 15 min at 37 °C to cross-link proteins and DNA. The cross-linking reaction was stopped with a 5-min treatment with 0.125 M glycine (final concentration) at room temperature. Cells were subsequently scraped off the Petri dish and they were washed and lysed by treatment with Nuclear LB {(50 mM Tris (pH 8.0), 10 mM EDTA, and 0.5% SDS) with added fresh 1× Halt™ Protease and Phosphatase Inhibitor Cocktails (Thermofisher, Cat. No 78444)} for 10 min on ice. Cellular lysates were diluted with IP Dilution buffer (16.7 mM Tris (pH 8.0), 167 mM NaCl, 1.2 mM EDTA, 1.1% Triton X-100, and 0.01% SDS) to a final volume of 1 mL and sonicated to shear the DNA to an average length of 300- to 500-bp fragments. Following sonication, the lysates were first centrifuged for 30 min at 18,000 g at 4 °C and the supernatants were incubated with protein A and salmon sperm DNA-bound agarose beads (Cell Signaling, Cat. No 9863), for 1 h at 4 °C. The precleared lysates were incubated overnight with the diluted primary antibody or with the Rabbit Isotype Control antibody (Thermofisher, Cat. No 10500 C) and following this, they were incubated with the Pierce™ Protein A/G Magnetic Beads (Thermofisher, Cat. No 88803) for 4 h at 4 °C. The immunoprecipitates were then washed sequentially with the following buffers. A Low Salt Wash Buffer {20 mM Tris (pH 8.0), 2 mM EDTA, 150 mM NaCl, 1% Triton X-100, and 0.1% SDS}, a High Salt Wash Buffer {20 mM Tris (pH 8.0), 2 mM EDTA, 500 mM NaCl, 1% Triton X-100, and 0.1% SDS}, a LiCl Wash Buffer {10 mM Tris (pH 8.0), 1 mM EDTA, 250 mM LiCl, 1% NP-40, and 1% (w/v) deoxycholic acid and TE buffer (10 mM Tris (pH 8.0), 1 mM EDTA}. The immunoprecipitated DNA was recovered by reversing the crosslinking with NaCl, and following incubation with proteinase K, it was extracted with DNA Purification Buffers and Spin Columns (Cell SIgnaling, Cat. No 14209). The immunoprecipitated DNA of the target loci, was then amplified by quantitative PCR, using the sets of primers listed in Supplementary Table 2 , the iTaq™ Universal SYBR® Green Super mix (Biorad, Cat No. 1725121) and a StepOne Plus qRT-PCR machine (Thermofisher). The same was done with input DNA, isolated from 2% of the pre-cleared nuclear lysate, prior to the immunoprecipitation. Fold enrichment was calculated, using the software https://www.sigmaaldrich.com/technical-documents/articles/biology/chip-qpcr-data-analysis.html ) provided online by Sigma-Aldrich. The detailed protocol can be found in the online protocol repository [85] . ChIP-seq: library preparation, sequencing, and analysis ChIP-seq libraries were generated using NEB Next® Ultra™ II DNA Library Prep Kit for Illumina® (New England Biolabs, Cat. no. E7645) and following the manufacturer’s protocol. ChIP-seq libraries were quality-checked using FastQC ( www.bioinformatics.babraham.ac.uk/projects/fastqc/ ). High-quality libraries were sequenced on an Illumina HiSeq 2500 platform. ChIP-seq experiments were performed in duplicate, and average depth of sequenced samples was 49 M (±5M) 100 bp paired-end reads. Sequencing results were demultiplexed with bcl2fastq. Compressed and demultiplexed fastq file pairs from each sample were used for analysis. Adapters and sequence contaminants were detected and removed using Cutadapt [77] . Paired-end reads were aligned against the human reference genome (GRCh38/hg38) using Bowtie (version 2.2.6) (with default parameters). Peak discovery was performed with HOMER (version 4.6) [86] . Sonicated input DNA was used as a control for peak discovery. Data snapshots were created using the Integrative Genomic Viewer of the Broad Institute ( https://software.broadinstitute.org/software/igv/home ) [87] . Sequencing was performed in the DNA sequencing Center of Brigham Young University (Provo, UTAH) ( https://biology.byu.edu/dnasc ). Chromatin immunocleavage (ChIC) [88] NCI-H1299 cells were FACS-sorted based on DNA content, as described above. Cell pools enriched for cells in G0/G1, S, and G2/M phase of the cell cycle (5 × 10 4 cells /pool) were washed multiple times with wash buffer (20 mM HEPES pH 7.5, 150 mM NaCl and 0.5 mM Spermidine, supplemented with fresh 1x Halt™ Protease and Phosphatase Inhibitor Cocktails). In parallel with the preparation of the cells, the antibodies to be used for ChIC (Supplementary Table 1 ) were attached to activated Magnetic Biomag Plus Concanavalin A Beads (Bangs Laboratories, Cat. No. BP531). To activate the Magnetic Biomag Plus Concanavalin A Beads (Bangs Laboratories, Cat. No. BP531), we washed the first multiple times with a binding buffer (20 mM HEPES-KOH, pH 7.9, 10 mM KCl, 1 mM CaCl 2 , and 1 mM MnCl 2 ). The activated beads were mixed with 50 μL of the primary antibody or Rabbit Isotype Control antibody (Thermofisher, Cat. No 10500C) diluted 1/50 in antibody buffer (2 mM EDTA (pH 8.0), 0.1% (wt/vol) digitonin diluted in wash buffer) and the bead-attached primary antibodies were mixed and incubated with the cell pellet at 4 °C overnight. The resulting immunoprecipitates were washed multiple times with wash buffer and then mixed with 50 μL of a 1/50 dilution of a Guinea Pig anti-Rabbit IgG (Heavy & Light Chain) secondary antibody (Antibodies-Online, Cat. No. ABIN101961) and incubated at 4 °C for 4 h. Following multiple washes, the immunoprecipitates were mixed with micrococcal nuclease (CUTANA™ pAG-MNase. EpiCypher, Cat No. SKU: 15-1116) (final concentration 700 ng/mL), which interacts with the ABIN101961 secondary antibody. The antibody-bound MNase was activated with the addition of 100 mM Ca 2+ (CaCl 2 ) and following activation, it digested the antibody-bound DNA in a reaction which was allowed to proceed for 30 min on ice. The reaction was terminated with the addition of 2× stop buffer (NaCl, 340 mM, EDTA 20 mM pH 8.0, EGTA 4 mM, digitonin 0.1% (wt/vol), RNAse A 0.2 mg, Glycogen 0.02 mg) and the chromatin fragments were released, following a 10-min incubation at 37 °C. Subsequently, the chromatin fragments were extracted using DNA Purification Buffers and Spin Columns (Cell SIgnaling, Cat. No 14209). DNA amplification by quantitative PCR, and data analyses were carried out as described under chromatin immunoprecipitation. RNA immunoprecipitation The first step in the RNA immunoprecipitation protocol was the cross-linking of proteins with DNA, which was carried out by treating the cells with 1% formaldehyde, as described under ChIP. Following cross-linking, the cells were scraped into 1 mL of Phosphate Buffered Saline (PBS)-Nuclear Isolation Buffer (sucrose 1.28 M, Tris-HCl 40 mM, MgCl 2 20 mM, and 4% Triton X-100) (ratio 1:1:3). Following this, the cells were washed twice and then lysed with RIP buffer (150 mM KCl, 25 mM Tris-HCl, 5 mM EDTA, 0.5 mM DTT, and 0.5% NP-40), supplemented with fresh 1× Halt™ Protease and Phosphatase Inhibitor Cocktails (Thermofisher, Cat. No 78444) and RNaseOUT™ Recombinant Ribonuclease Inhibitor (Thermo Fisher, Cat. No. 10777019) and the lysates were kept on ice for 10 min. Subsequently, the lysates were clarified by centrifugation at 18,400 x g at 4 °C for 30 min and a fraction of the supernatant was incubated with protein A and salmon sperm DNA-bound agarose beads (Cell Signaling, Cat. No 9863), for 1 h in 4 °C. The clarified lysates were then incubated with the immunoprecipitating antibody or an isotype control antibody (rabbit isotype control-Thermofisher, Cat. No 10500 C or mouse isotype Control-Thermofisher, Cat. No 10400C) at 4 °C overnight. The resulting antigen–antibody complexes were incubated with Pierce™ Protein A/G Magnetic Beads (Thermofisher, Cat. No 88803) at 4 °C for 4 additional hours and the immunoprecipitates were washed four times using the RIP buffer. The RNA–protein complexes were eluted in 100 μL of RIP buffer and the RNA was recovered by reverse cross-linking at 70 °C and proteinase K incubation at 55 °C. The RNA was then extracted with phenol–chloroform–isoamyl alcohol and it was precipitated with ethanol at -80 °C overnight, in the presence of yeast tRNA carrier (10 mg/mL). The immunoprecipitated RNA fragments and input RNA derived from clarified cell lysates corresponding to 2% of the amount of lysate used for RNA IP were reverse-transcribed with random hexamers. The abundance of the amplified RNA fragment in the two pre-mRNA-derived pools was measured by quantitative RT-PCR, carried out in triplicate. The primer sets used in these amplification reactions correspond to intronic and exonic regions of target pre-mRNAs. Amplification reactions were carried out, using the iTaq™ Universal SYBR® Green Super mix (Biorad, Cat No. 1725121) and a StepOne Plus qRT-PCR machine (Thermofisher). The data were analyzed using software provided online by Sigma-Aldrich. ( https://www.sigmaaldrich.com/technical-documents/articles/biology/chip-qpcr-data-analysis.html ). SNRNP-70 binding in the human U1 snRNP gene, using the primers F: 5′-GGG AGA TAC CAT GAT CAC GAA GGT-3′, R: 5′-CCA CAA ATT ATG CAG TCG AGT TTC CC-3′, was used as the control for RNA IPs. The detailed protocol can be found in the online protocol repository [85] . Tumor xenografts Ethics statement All mouse experiments were approved by the Institutional Animal Care and Use Committee (IACUC) of the Ohio State University. IACUC protocol number 2018A00000134, PI: Philip N. Tsichlis Experimental protocol A total of 2 × 10 6 NCI-H1299 cells, 5 × 10 6 A549 cells, and 1 × 10 7 NCI-H1975 cells were suspended into 30% Matrigel (Corning, Cat. No. 356231) in PBS in a total volume of 200 µL and implanted subcutaneously into the flanks of 6-week-old NSG ( NOD.Cg-Prkdc scid -IL2rg tm1Wjl /Scj ) mice (left side for the shControl and right side for the shIWS1 cells). The mice were monitored every 3 days and the size of the tumors was measured using a digital caliper. The tumor volume was calculated with the modified ellipsoid formula: \(V=\frac{1}{2}\nu \times {{{s}^{2}}^{}}^{}\) (where v is length and s is width). The mice were sacrificed 4 weeks (NCI-H1299 and NCI-H1975 cells), or 6 weeks (A549 cells) post inoculation. Tumors were resected and their weights were measured. Part of each resected tumor was snap-frozen in liquid nitrogen and was kept at −80 °C for RNA and protein isolation. The remainder was fixed in 10% (v/v) formalin (Sigma, Cat. No. HT501640) overnight. Subsequently, it was transferred to 70% EtOH and following this, it was embedded in paraffin at the Comparative Pathology & Mouse Phenotyping Shared Resource of the OSUCCC, prior to H and E and immunohistochemistry (IHC) staining. RNA and protein isolation from mouse xenografts About 50–100 mg of the frozen mouse xenografts were homogenized in 1 mL of Trizol reagent (Thermofisher Scientific, Cat. No. 15596026). RNA and protein were isolated from the homogenized samples by following the instructions of the manufacturer. Briefly, 200 µL of chloroform (Sigma, Cat. No. C2432) were added to all the 1 mL Trizol extracts and following mixing, the extracts were centrifuged at 12,000 × g for 15 min at 4 °C for phase separation. Following this, the RNA in the aqueous phase was transferred into a new tube, while the organic phase was stored O/N at 4 °C for protein isolation. RNA extraction RNA was precipitated by mixing the aqueous phase with 0.5 mL of isopropanol (Fisher Scientific, Cat. No. A416P-4). Following incubation at RT for 15 min, the aqueous phase/isopropanol mixture was spun at 12,000 × g for 10 min at 4 °C. The RNA pellet was washed with 75% ethanol, followed by a second spin at 7500 × g for 5 min at 4 °C and was dissolved in 30 µL of DEPC-treated water (IBI Scientific, Cat. No. IB42210). Protein extraction About 0.3 mL of 100% ethanol was added to the interphase–organic phase and the samples were centrifuged at 2000 × g for 5 min at 4 °C. The proteins in the phenol–ethanol supernatant were then precipitated by adding 1.5 mL of isopropanol, followed by incubation at room temperature for 10 min and centrifugation at 12,000 × g at 4 °C for 10 min. The protein pellet was washed 3 times in a solution of 0.3 M guanidine hydrochloride (Sigma, Cat. No. SRE0066) in 95% ethanol. Each wash cycle included the resuspension of the pellet in the wash solution, a 20-min incubation at room temperature, and centrifugation at 7500 × g at 4 °C for 5 min. After the final guanidine hydrochloride wash, the pellet was washed again, in 100% ethanol, the ethanol resuspended pellet was incubated for 20 min at room temperature, and was centrifuged at 7500 × g for 5 min at 4 °C. The protein pellet was dissolved in 200 µL of 1% SDS, supplemented with a protease and phosphatase inhibitor cocktail (Thermo Fisher Scientific, Cat. No. 78444). Insoluble material was removed by centrifugation at 10,000 × g for 10 min at 4 °C. Cellular protein and RNA were analyzed by immunoblotting and qRT-PCR, respectively. The antibodies and primers we used for these analyses are listed Supplementary Tables 1 and 2 . IHC staining About 5-μm-thick sections of the paraffin-embedded mouse tumors were heated to 55 °C for 20 min prior to deparaffinization with xylene (Fisher scientific, Cat. No. X3F-1GAL). Following deparaffinization, tissue sections were rehydrated by treatment with decreasing concentrations of ethanol, down to distilled water. The endogenous peroxidase activity was blocked by treatment with 3% H 2 O 2 (Fisher Scientific, Cat. No. H325500) in PBS (pH 7.4), at room temperature for 10 min. This was followed by antigen retrieval via a 30-min treatment at 80 °C, with Citrate Buffer, pH 6.0, Antigen Retriever (Sigma, Cat. No. C9999). Subsequently, tissues were rinsed with PBS for 5 min and then treated with normal goat blocking serum at room temperature for 20 min. Subsequent steps were carried out using the Vectastain Elite ABC Universal kit peroxidase (Vector Laboratories, Cat. No. PK-6200). Briefly, following treatment with the blocking serum, and a 5-min wash with PBS at room temperature, the tissues were incubated with the primary antibody diluted in PBS with 2.5% serum at 4 0 C overnight. Subsequently, the tissues were rinsed with PBS for 5 min at room temperature, and incubated with the biotinylated Universal Antibody for 30 min, also at room temperature. Following an additional single, room-temperature 5-min wash with PBS, the tissues were treated with the Vectastain Elite ABC reagent for 30 min at room temperature, to enhance the signal. An additional single 5-min wash with PBS was followed by a 2–10 min incubation with a DAB peroxidase substrate solution (Vector Laboratories, Cat. No. SK-400) according to the manufacturer’s instructions. At the end, the slides were washed with tap water and covered with the DPX mounting medium (Sigma, Cat. No. 06522). The primary antibodies used for staining are listed in Supplementary table 1 . All IHC images were captured on a Nikon eclipse 50i microscope with attached Axiocam 506 color camera using the ZEN 2.6 blue edition software (Zeiss). Imaging files were imported to ImageJ [89] for analysis. Using the native freehand function of the software, the signal derived from glandular areas of the tumor was measured and was divided by the surface area occupied by these glandular areas. For each sample, at least five different sections of the tumor were scanned. The final score for each tumor was the average value of these measurements. To ensure that the analysis was unbiased, the protocol described above was followed for the analysis of all the images generated in the course of all the experiments in this report. Human tumor samples Tumor procurement and analysis Thirty LUAD samples with matching NAT were obtained from the Tissue Bank of The Ohio State University, under the universal consenting and biobanking protocol, Total Cancer Care (TCC). TCC is the single protocol used by the Oncology Research Information Exchange Network (ORIEN), which was formed through a partnership between OSUCCC-James and the Moffitt Cancer Center (Tampa, FL). For more information, please see the Biospecimen Core Services facility of The Ohio State University Comprehensive Cancer Center ( https://cancer.osu.edu/for-cancer-researchers/resources-for-cancer-researchers/ shared-resources/biospecimen-services) and the ORIEN project ( https://cancer.osu.edu/for-cancer-researchers/resources-for-cancer-researchers/orien ). Ten additional consented LUADs without matching normal tissue had been obtained earlier from the tissue bank of Tufts Medical Center. The latter had also been used in an earlier study on the role of IWS1 in NSCLC (Sanidas et al. [22] ). All tumor samples were provided to this study as unidentified samples. Frozen tissues were grinded on dry ice into very small pieces, which were then transferred into chilled 2-mL round-bottom Eppendorf tubes. Protein was extracted by adding 500 μL of ice-cold NP-40 LB (50 mM Tris-HCl, pH 7.5, 150 mM NaCl, 0.5% Triton X, and 1 mM EDTA, pH 8, supplemented with a protease and phosphatase inhibitor cocktail (Thermo Scientific Cat Nr 78442)) followed by homogenization of the tissue fragments with an electric homogenizer, on ice. Homogenized samples were moved into chilled microcentrifuge tubes, kept for 40 min on ice, and then centrifuged at 16,000x g for 20 min at 4 °C. Supernatants were collected in fresh tubes and placed on ice for protein quantification, which was performed using the BioRad Bradford Reagent (Biorad, Cat. No. 5000001). RNA was extracted by grinding tissue samples as before, in 1 mL Trizol Reagent (Thermo Fisher, Cat. No. 15596026) and by following the manufacturer’s instructions for subsequent extraction steps. IHC staining of lung adenocarcinomas was done using lung adenocarcinoma tissue arrays (US Biomax, LC1504). The staining procedures and the analysis of the data were done as described for the mouse xenografts. Since the tissue arrays contain only two sections from each tumor, the final score for a given tumor was the average of the scores for the two sections. Data analysis Western blot images were imported to ImageJ and the intensity of the bands was measured. The values obtained from this analysis were normalized to tubulin and the normalized values were imported to GraphPad Prism 8.4. Correlation coefficients were calculated using simple linear regression. Following this, correlations were visualized in heatmaps. The exact values and statistical significance of the correlations can be found in Supplementary Table 5 . The U2AF2 E2/E3 ratios, generated from the analysis of the RNAs of the 40 LUADs in our patient cohort and the quantitative data generated from the IHC analyses of the tissue microarrays were also imported in Image J and they were analyzed and presented as described for the western blot data. The exact values and statistics of the correlation analyses, can also be found in Supplementary Table 5 . The information available for all the lung adenocarcinomas in our cohort included sex, age, and clinical stage, and the information available for the tissue array cohort, included clinical stage and histologic grade. For the 30 OSU tumor samples, patient survival was also available. All the tumors in our cohort were also analyzed for EGFR and KRAS genetic alterations and, based on this analysis, they were subclassified into EGFR mutant and KRAS mutant subgroups. As mentioned in the preceding paragraph, western blot and IHC data were quantified by Image J and following normalization, they were imported into GraphPad Prism 8.4. The first question we addressed was whether the pathway we defined with controlled experiments in cultured cells was also active in naturally occurring human lung adenocarcinomas. This was addressed by measuring the correlation coefficients between IWS1 and phosphor-IWS1 and multiple mediators and targets of the pathway, as described in the preceding paragraph. The correlations were presented in heatmaps and although correlations were observed in all the tumors, they were significantly more robust in EGFR mutant tumors. To determine the clinical importance of the IWS1 phosphorylation pathway, we examined the activity of the pathway in Stage I vs Stage II/III tumors and in Grade 2 vs Grade 3 tumors. The surrogate markers for the activity of the pathway were the levels of phosphor-IWS1 and the U2AF2 E2/E3 ratio, both of which were quantified and imported to GraphPad Prism 8.4, as described in the preceding paragraph. To determine whether the activity of the pathway impacts patient survival, we divided the tumors in our cohort into high and low phosphor-IWS1 tumors and into high and low U2AF2 E2/E3 ratio tumors. Survival curves of tumors in the high and low categories were generated, using the Kaplan–Meir method [90] and they were statistically compared using the log-rank test. A tumor was identified as a high IWS1 or high E2/E3 ratio tumor, if the value of these parameters in the given tumor was higher than the mean value, plus one standard deviation over the mean (mean+ 1 SD). All tumors below this mark were classified as low phosphor-IWS1, or as low U2AF2 E2/E3 ratio tumors. Publicly available LUAD datasets and analyses The Cancer Genome Atlas (TCGA) dataset TCGA data were downloaded from https://portal.gdc.cancer.gov/ . Overall, 658 TCGA-LUAD patients (all stages), 162 TCGA-LUAD (all stages) with KRAS mutations, and 67 TCGA-LUAD with EGFR mutations were obtained with their survival and clinical data (clinical stage, metastasis, and survival). A total of 516 out of 658 had RNA-seq data. For the expression of SRSF1, 128 out of 658 had RNA-Seq data. Figures for the correlation analysis were generated using the visualization tools of the Xena browser ( http://xena.ucsc.edu/ .) and GraphPad Prism 8.4. The clinical stage and Metastasis analysis for the TCGA-LUAD patients was performed as described above. 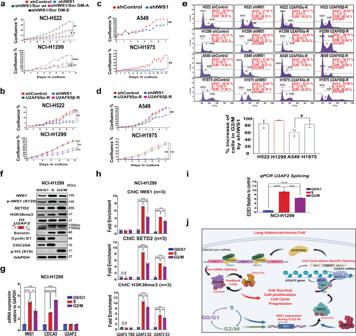The Survival analysis was performed in GraphPad Prism 8.4 with a Kaplan–Meier method and log-rank p statistics, with similar approach to the cut-off decision as described above. Gene Expression Omnibus (GEO) repository datasets GSE141685 This dataset includes RNA-Seq data of brain metastases derived from six LUAD patients, and 24 primary nonmetastatic LUADs, independent of stage and mutational status (12 early- and 12 late- stage LUADs). Fig. 6: IWS1 phosphorylation promotes cell proliferation by controlling a Sororin/ERK phosphorylation feedback loop, throughU2AF2RNA splicing. a,bGrowth curves of shControl and shIWS1 NCI-H522 and NCI-H1299 cells, growing in fully supplemented media, before and after rescue with Sororin (wt or mutants), or U2AF65α/U2AF65β. Experiment was done in triplicate and proliferation was expressed as mean percent confluence ±SD.Pvalues (one-sided unpairedt-test) were calculated for the endpoint measurements. *p< 0.05, **p< 0.01, ***p< 0.001, ****p< 0.0001.bGrowth curves of shControl and shIWS1 A549 and NCI-H1975 cells.cGrowth curves of the same shIWS1 cells rescued with U2AF65α or U2AF65β. Proliferation in panelscanddwas measured as in panelsaandb.d(Upper panel) Cell cycle profiles of the indicated propidium iodide (PI)-stained cell lines. One representative, out of three biological replicates. Mean percentages of cells in different cell cycle phases in red. (Lower panel) shIWS1-induced percent change of cells in G2/M±SD. Statistical analysis was performed using a one-sided unpairedt-test, *p <0.05. Gating strategy in supplementary figure 8a.eNCI-H1299 cells were sorted into G0/G1, S and G2/M fractions. Lysates of sorted cells were probed with the indicated antibodies. RT-PCR on RNA from the same cells, using primers forU2AF2exons 1 and 3. Gating strategy in supplementary figure 8a.fqRT-PCR-determined expression ofIWS1,CDCA5andU2AF2, relative to GAPDH±SD. SD was calculated based on three biological replicates.gChIC-determined mean fold enrichment of IWS1, SETD2 and H3K36me3 in cell cycle fractionated cells in the indicated regions of theU2AF2RNA±SD.hqRT-PCR-based calculation of the meanU2AF2 E2/E3ratio in S and G2/M, relative to G0/G1 cells ±SD. SD was calculated based on three biological replicates *p< 0.05, **p< 0.01, ***p< 0.001, ****p< 0.0001. (one-sided unpairedt-test).iIWS1 expression is induced during the S and G2/M phases of the cell cycle. Following phosphorylation by AKT3, IWS1 orchestrates the cell cycle-dependent assembly of epigenetic complexes on theU2AF2gene. This promotes the inclusion of exon 2 in theU2AF2mRNA. U2AF65α, encoded by the exon 2-containingU2AF2mRNA, interacts with Prp19, promotingCDCA5splicing and the expression of Sororin. The latter is phosphorylated by ERK, and promotes ERK phosphorylation, in a positive feedback loop, which stimulates proliferation of lung adenocarcinomas. The primary LUADs were obtained from the TCGA dataset and the TCGA ID of these patients, along with their clinical information are presented in Supplementary Table 6 . The FPKM (fragments per kilobase per million fragments) values were downloaded for further analysis. First, we compared the IWS1 FPKM values in the primary tumors and the metastatic lesions and we presented them in violin plots. Next, we calculated the U2AF2 E2/E3 and the FGFR2 E8/E9 ratios, as described under the TCGA dataset and we presented them also in violin plots. Using GraphPad Prism 8.4, we visualized FPKM values of genes in the IWS1 pathway in the primary tumors and the metastatic lesions, as heatmaps. The exon expression profiles of the TCGA and GSE141685 LUAD samples were measured experimentally using the Illumina HiSeq 2000 RNA Sequencing platform. Exons were mapped to the human genome, using UCSC Xena unc_RNAseq_exon probeMap. Exon-level transcription estimation was presented in RPKM values (reads per kilobase per million mapped reads). A log 2 (RPKM+1) exon expression matrix was then imported to the RStudio framework (V 3.5.2) for the selection and export of the values of exons 2 and 3 of U2AF2 and exons 8 and 9 of FGFR2 . GSE13213 [70] A LUAD gene expression dataset, based on the Agilent microarray technology. In total, 117 tumors were divided into two groups, one with high ( n = 59) and another one with low ( n = 58) probability of relapse. Fourteen of these tumors harbored KRAS mutations and 45 harbored EGFR mutations. To determine the significance of the IWS1 phosphorylation pathway in tumor relapse, we examined the expression of IWS1, Sororin, CDK1, and Cyclin B1 in patients with high and low probability of relapse. Data were presented as heatmaps, which were generated, using GraphPad Prism 8.4. GSE26939 [91] A LUAD gene expression dataset based on the Agilent microarray technology. The microarray data of individual tumors were linked to patient survival data. Based on the microarray data and using the criteria described under “data analysis” in the “human tumor samples” section, tumors were first placed into high or low IWS1 subgroups. The low IWS1 subgroup contained 17 tumors with a KRAS mutation and 27 tumors with an EGFR mutation and the high IWS1 subgroup contained 18 tumors with a KRAS mutation and 26 with an EGFR mutation. Survival curves of patients with low and high IWS1 tumors were generated, using the Kaplan–Meier methodology and Log-rank statistics. Gene expression values in Agilent two color arrays were expressed as the log 2 ratios of the two color signals. These normalized and background-corrected values were imported from the microarray dataset into the RStudio-integrated development environment (IDE) (V 3.5.2) for analysis. Log 2 ratios for IWS1 , CDCA5 , CDC2 , and CCNB1 were exported from the RStudio IDE into an Excel file and they were used to generate heatmaps, violin plots, or Kaplan–Meier survival curves. GSE123903 [71] A set of single-cell RNA-Seq (scRNA-seq) data derived from the analysis of tumor cells from a patient-derived LUAD mouse model. The normalized scRNA-seq counts were retrieved and analyzed for IWS1 and CDCA5 expression. The data were visualized using the Barnes–Hut approximate version of t-SNE [92] ( https://github.com/lvdmaaten/bhtsne ). Statistics and reproducibility The experiments in Fig. 1f–g and Supplementary Figs. 1e –i; 2a –c; 3a –d, a–c; 4a –c, a–g; 5a –g, b–h; 6a –d, a–i; 7a –f; 8b , c; 9a, b were performed in a minimal of three independent biological experiments. The data in Fig. 7 (mouse xenografts) were performed once, using five mice/group. Western blots of the LUAD samples in 8a was performed two times. The IHC staining experiments of the mouse xenografts in Supplementary Fig. 10c and of the human tissue arrays, were performed once, using the antibodies and techniques listed in the Methods section. All the attempts at replications were successful. Statistical analyses were done using GraphPad Prism 8.4. All the statistical analyses can be found in the Mendeley dataset where the source data of this report were deposited [93] . Reporting summary Further information on research design is available in the Nature Research Reporting Summary linked to this article.